Polyploidy, regular patterning of genome copies, and unusual control of DNA partitioning in the Lyme disease spirochete 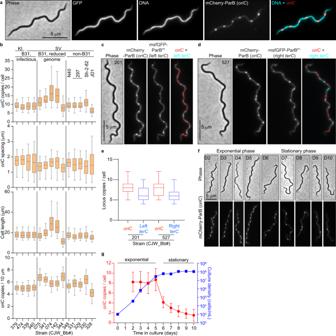Fig. 1:B. burgdorfericells contain multiple chromosome copies. aImages of a cell of strain CJW_Bb474 expressing cytosolic free GFP and mCherry-ParB. Hoechst 33342 was used to stain the DNA.bPopulation quantifications of exponentially growing cultures of the strains shown in Supplementary Fig.1c. Top to bottom: copy numbers per cell of the labeledoriCloci;oriCspacing (distances between adjacentoriCspots); cell lengths; andoriCdensities (copies per 10 μm of cell length). Strain numbers are indicated at the bottom. Shown are the mean of the data (middle line), the 25 to 75 percentiles of the data (box), and the 2.5 to 97.5 percentiles of the data (whiskers). Strain backgrounds andoriClabeling method (mcherry-parBknock-in, KI, or taggedparBexpressed from a shuttle vector, SV) are listed at the top.cPhase-contrast and fluorescence micrographs of a cell of strain CJW_Bb201, which expresses labels fororiC(mCherry-ParB) and the leftterClocus (msfGFP-ParBP1), respectively.dPhase-contrast and fluorescence micrographs of a cell of strain CJW_Bb527, which expresses labels fororiC(mCherry-ParB) and the rightterClocus (msfGFP-ParBP1), respectively. d and e. Images were acquired while the cultures were growing exponentially.eBoxplots oforiCandterCcopies per cell in exponentially growing cultures of strains CJW_Bb201 and CJW_Bb527. Shown are the mean of the data (middle line), the 25 to 75 percentiles of the data (box) and the 2.5 to 97.5 percentiles of the data (whiskers).fAn exponentially growing culture of strain CJW_Bb339, in whichoriCis labeled by expression of mCherry-ParB, was diluted to 103cells/mL then imaged daily from day 2 through day 10 of growth in culture. Shown are representative images of cells from the days indicated on the phase-contrast images.gPlot showing theoriCcopy number per cell (red, mean ± standard deviation) and the culture density (blue, in cells/mL) over time for the population imaged in (f). Source data for panels (b,e, andg) are provided as a Source Data file. The numbers (n) of cells analyzed and the number of replicates are provided in Supplementary Data2. 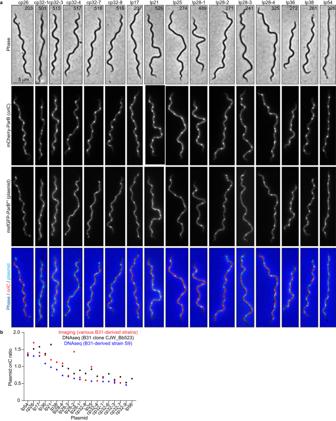Fig. 2: Exponentially growingB. burgdorfericultures contain multiple copies per cell of their endogenous plasmids. aImages of representative cells of strains in which theoriCloci were labeled by expression of mCherry-ParB while the plasmid indicated at the top was labeled by insertion of aparSP1sequence and expression of msfGFP-ParBP1. CJW_Bb strain numbers are marked on the phase-contrast images.bPlot showing the plasmid-to-oriCcopy number ratios determined by imaging the strains shown in (a) (red), or by marker frequency analysis of whole genome sequencing data (see methods) in strains S9 (blue) or strain CJW_Bb523, a clone of strain B31MI (black). Source data are provided as a Source Data file. The numbers (n) of cells analyzed and the number of replicates are provided in Supplementary Data2. Borrelia burgdorferi , the tick-transmitted spirochete agent of Lyme disease, has a highly segmented genome with a linear chromosome and various linear or circular plasmids. Here, by imaging several chromosomal loci and 16 distinct plasmids, we show that B. burgdorferi is polyploid during growth in culture and that the number of genome copies decreases during stationary phase. B. burgdorferi is also polyploid inside fed ticks and chromosome copies are regularly spaced along the spirochete’s length in both growing cultures and ticks. This patterning involves the conserved DNA partitioning protein ParA whose localization is controlled by a potentially phage-derived protein, ParZ, instead of its usual partner ParB. ParZ binds its own coding region and acts as a centromere-binding protein. While ParA works with ParZ, ParB controls the localization of the condensin, SMC. Together, the ParA/ParZ and ParB/SMC pairs ensure faithful chromosome inheritance. Our findings underscore the plasticity of cellular functions, even those as fundamental as chromosome segregation. Lyme disease is the most prevalent vector-borne infectious disease in North America and Europe [1] . Its geographic range has steadily spread over the years, with caseloads recently estimated to be near 500,000 per year in the United States [1] , [2] . Lyme disease is caused by Borrelia burgdorferi and related spirochete bacteria [3] . In nature, Lyme disease spirochetes undergo a transmission cycle between Ixodes hard tick vectors and warm-blooded vertebrate hosts [4] . Infection in humans via a tick bite can result in a wide variety of symptoms when left untreated. Disease manifestations range from skin rashes, fever, and malaise during early stages of the disease to arthritis, carditis, and neurological symptoms during later stages [3] . Given B. burgdorferi ’s medical relevance, we set out to study basic biological processes necessary for cell proliferation. This topic is of considerable interest because bacterial multiplication is a prerequisite for successful transmission, host infection, and disease causation. B. burgdorferi was identified in 1982 [5] . Despite four decades of research, many of the fundamental cellular processes underlying the ability of this bacterium to self-replicate remain understudied. This is in part because B. burgdorferi has a long doubling time (5 to 18 h) in culture [6] , [7] , [8] , [9] , [10] , [11] . Additionally, genetic manipulation of this organism, while possible [12] , [13] , [14] , remains challenging compared to that of Escherichia coli and other common model bacteria. However, knowledge obtained from the study of model bacteria does not always translate to unrelated species, including spirochetes. These bacteria form a phylum of particular interest because, in addition to B. burgdorferi , it includes important human pathogens such as the agents of relapsing fever, syphilis, and leptospirosis. In this study, we focused on one of the most enigmatic and important aspects of B. burgdorferi’s biology: genome inheritance. Faithful genome inheritance during cellular replication is essential for the propagation of all life forms. Despite its small size of ~1.5 megabases [15] , the B. burgdorferi genome is the most segmented bacterial genome known to date [16] . It is composed of one linear chromosome and over 20 linear or circular plasmids, several of which have essential roles during the spirochete’s natural tick-vertebrate transmission cycle [4] , [15] , [17] , [18] . Quantitative polymerase chain reaction (qPCR)-based measurements [19] generated the common (though not universal [20] ) view that B. burgdorferi has about one chromosome copy per cell. Endogenous plasmids have between one and three times the copy number of the chromosome [21] , [22] , [23] , [24] , [25] . Given the large size of B. burgdorferi cells (10 to 25 µm or longer depending on the strain) [26] , [27] , [28] , monoploidy means that the replicated chromosome and plasmids would have to segregate over long distances to ensure their faithful inheritance during division. This, however, has not been examined experimentally. Experiments in a heterologous E. coli system, together with a transposon screen in B. burgdorferi , have suggested that the replication and partitioning of B. burgdorferi plasmids are mediated by specific plasmid-encoded proteins via unknown mechanisms [18] , [29] , [30] , [31] . On the other hand, chromosome segregation is predicted to involve a ParA/ParB system [15] , [32] . ParA and ParB proteins are well known to work together to mediate the segregation of duplicated chromosomal origins of replication ( oriC ) in broadly diverse bacteria [32] , [33] . ParB is often referred to as a “centromere-binding” protein because it specifically binds to centromere-like sequences ( parS ) usually located near oriC [32] . After loading on the DNA at the parS sites, ParB spreads onto adjacent sequences [34] , [35] , [36] to form a partition complex. ParA is an ATPase that dimerizes upon ATP binding, which in turn promotes the nonspecific binding of the ParA dimer to the DNA (the nucleoid) [37] , [38] . Upon interaction with ParA, the ParB-rich partition complex stimulates the ATPase activity of ParA, causing dimer dissociation and release of ParA from the DNA [38] , [39] . Repetition of this biochemical cycle, combined with a translocation force [40] derived from the elastic properties of the chromosome [41] , [42] , [43] , [44] and/or a diffusion-based mechanism [45] , [46] , [47] , [48] , drives the translocation and therefore the segregation of replicated partition complexes [33] , [49] . The B. burgdorferi chromosome contains a parS site [32] near oriC and encodes both ParA and ParB homologs [15] , predictive of a conserved ParA/ParB function in chromosome segregation. In this study, we genetically labeled and imaged various chromosomal loci and plasmids in live B. burgdorferi cells. Fluorescence microscopy analysis, combined with genetic deletions and ChIP-seq experiments, revealed that B. burgdorferi is polyploid and uses a novel centromere-binding protein, rather than ParB, to carry out a key DNA partitioning activity. B. burgdorferi cells carry multiple chromosome copies during growth To label oriC in live B. burgdorferi cells, we relied on the specific recognition of the oriC -proximal parS site by ParB (see Supplementary Notes and Supplementary Fig. 1a, b ). We therefore substituted the parB gene with mcherry-parB at the endogenous locus. The resulting strain (CJW_Bb474), which also expressed free GFP for cytoplasm visualization, was stained with the Hoechst dye to reveal DNA localization. In this strain, we would expect one or two fluorescent mCherry-ParB puncta within the nucleoid to reflect a monoploid state before and after initiation of chromosomal DNA replication, respectively. However, each cell had multiple mCherry-ParB foci that appeared regularly spaced along the nucleoid (Fig. 1a ). Fig. 1: B. burgdorferi cells contain multiple chromosome copies. a Images of a cell of strain CJW_Bb474 expressing cytosolic free GFP and mCherry-ParB. Hoechst 33342 was used to stain the DNA. b Population quantifications of exponentially growing cultures of the strains shown in Supplementary Fig. 1c . Top to bottom: copy numbers per cell of the labeled oriC loci; oriC spacing (distances between adjacent oriC spots); cell lengths; and oriC densities (copies per 10 μm of cell length). Strain numbers are indicated at the bottom. Shown are the mean of the data (middle line), the 25 to 75 percentiles of the data (box), and the 2.5 to 97.5 percentiles of the data (whiskers). Strain backgrounds and oriC labeling method ( mcherry-parB knock-in, KI, or tagged parB expressed from a shuttle vector, SV) are listed at the top. c Phase-contrast and fluorescence micrographs of a cell of strain CJW_Bb201, which expresses labels for oriC (mCherry-ParB) and the left terC locus (msfGFP-ParB P1 ), respectively. d Phase-contrast and fluorescence micrographs of a cell of strain CJW_Bb527, which expresses labels for oriC (mCherry-ParB) and the right terC locus (msfGFP-ParB P1 ), respectively. d and e. Images were acquired while the cultures were growing exponentially. e Boxplots of oriC and terC copies per cell in exponentially growing cultures of strains CJW_Bb201 and CJW_Bb527. Shown are the mean of the data (middle line), the 25 to 75 percentiles of the data (box) and the 2.5 to 97.5 percentiles of the data (whiskers). f An exponentially growing culture of strain CJW_Bb339, in which oriC is labeled by expression of mCherry-ParB, was diluted to 10 3 cells/mL then imaged daily from day 2 through day 10 of growth in culture. Shown are representative images of cells from the days indicated on the phase-contrast images. g Plot showing the oriC copy number per cell (red, mean ± standard deviation) and the culture density (blue, in cells/mL) over time for the population imaged in ( f ). Source data for panels ( b , e , and g ) are provided as a Source Data file. The numbers ( n ) of cells analyzed and the number of replicates are provided in Supplementary Data 2 . Full size image We confirmed this finding in 13 additional B. burgdorferi strains derived from different lineages of the strain B31, or from other B. burgdorferi isolates, including the well-studied N40 and 297 strains (Fig. 1b and Supplementary Fig. 1c ; also see Supplementary Notes for strain construction and oriC labeling). The spacing between adjacent oriC copies was similar across all tested strains (Fig. 1b ). As a complementary approach, we labeled the oriC -proximal uvrC locus of the B. burgdorferi B31 chromosome with the orthogonal msfGFP-ParB P1 / parS P1 pair derived from the E. coli P1 plasmid and observed similar results (see Supplementary Notes and Supplementary Fig. 1a, b, d–f ). To demonstrate that the detection of multiple oriC copies reflects the presence of multiple chromosomes per cell, we genetically labeled and visualized the left and right telomeres ( terC ) using the msfGFP-ParB P1 / parS P1 system (Fig. 1c–e ). We also confirmed the presence of multiple terC copies per cell by DNA fluorescence in situ hybridization (Supplementary Fig. 1g ). Collectively, our data show that B. burgdorferi cells contain multiple complete chromosomes and thus are polyploid during exponential growth in culture. We found that the discrepancy between our polyploidy results and previous qPCR measurements of ~1.3 chromosomes per cell [19] stemmed from a difference in the culture growth stage. While we imaged cultures in exponential growth (Fig. 1a–e , Supplementary Fig. 1b–g ), the previous analysis was done using saturated cultures [19] , which had likely reached stationary phase. Indeed, we found that the oriC copy number decreases in stationary phase cultures, ultimately reaching about one copy per cell (Fig. 1f, g ). qPCR measurements of chromosomal copies in different growth stages confirmed that exponentially growing cells contain multiple chromosome copies and that their copy numbers decrease in the stationary phase (Supplementary Fig. 1h ), in agreement with our imaging results (Fig. 1f, g ). In fact, these findings are conceptually consistent with a previous study by Ornstein and Barbour [20] . B. burgdorferi cells contain multiple copies of their endogenous plasmids Next, we examined the localization and copy number of 16 distinct plasmids relative to the chromosome by generating different strains, each with a distinct endogenous plasmid labeled in addition to the oriC locus (Fig. 2a , Supplementary Data 1 ). For each plasmid, we detected multiple copies per cell (Fig. 2a , Supplementary Fig. 2a ). The plasmid: oriC ratios varied between ~0.5 and ~1.8 (Fig. 2b , Supplementary Fig. 2a ), which overlaps with previous findings that documented plasmid to chromosome copy number ratios between 1:1 and 3:1 [21] , [22] , [23] , [25] . These results were further confirmed by marker frequency analysis using whole genome sequencing (see methods) (Fig. 2b ). Moreover, the plasmids were regularly spaced within the cells (Fig. 2a ). As with the chromosome, the copy number of cp26 (Supplementary Fig. 2b ), and presumably that of the other plasmids, decreased as the axenic culture advanced into stationary phase, suggesting a potential coordination between independent segments of the genome. Fig. 2: Exponentially growing B. burgdorferi cultures contain multiple copies per cell of their endogenous plasmids. a Images of representative cells of strains in which the oriC loci were labeled by expression of mCherry-ParB while the plasmid indicated at the top was labeled by insertion of a parS P1 sequence and expression of msfGFP-ParB P1 . CJW_Bb strain numbers are marked on the phase-contrast images. b Plot showing the plasmid-to- oriC copy number ratios determined by imaging the strains shown in ( a ) (red), or by marker frequency analysis of whole genome sequencing data (see methods) in strains S9 (blue) or strain CJW_Bb523, a clone of strain B31MI (black). Source data are provided as a Source Data file. The numbers ( n ) of cells analyzed and the number of replicates are provided in Supplementary Data 2 . Full size image B. burgdorferi cells in fed nymphs are also polyploid While the phenotypes of stationary phase cultures were interesting (and will be explored in a separate study), we chose to focus our attention on B. burgdorferi during growth because cell proliferation is required for disease to occur. Outside the laboratory, B. burgdorferi cannot grow as a free-living organism. Therefore, to test whether the polyploidy observed in growing cultures has physiological relevance in a natural context, we colonized ticks with strain CJW_Bb474 expressing mCherry-ParB and cytoplasmic GFP through feeding on infected mice. 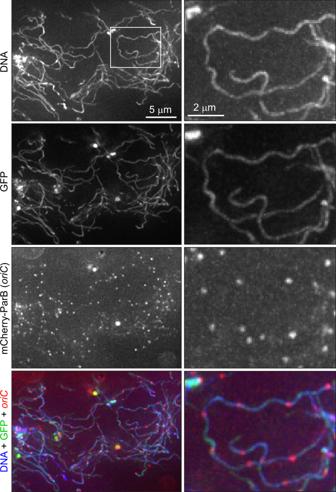Fig. 3: Tick-borneB. burgdorfericells contain multiple chromosome copies. Images of cells of strain CJW_Bb474 in the midgut of a nymphal tick 10 days after feeding drop-off. DNA was stained with Hoechst 33342. The mCherry-ParBoriCsignal was amplified by staining with RFP booster. Shown are max-Z projections of a deconvolved stack of images (left) and higher-magnification views of the region indicated by the white rectangle (right). This strain displayed no apparent defect in mouse infectivity either by needle injection or tick bite, or in acquisition by ticks feeding on infected mice (Supplementary Fig. 1i–k and Supplementary Notes ). Using three-dimensional deconvolution of image stacks, we were able to readily detect GFP-positive spirochetes in the midgut of fed, CJW_Bb474-colonized nymphs (Fig. 3 ). These spirochetes, which were co-stained with the DNA dye Hoechst, contained regularly spaced mCherry-ParB foci (Fig. 3 ). The complex three-dimensional orientation of the thin spirochetes within the tick midgut [50] prevented us from accurately determining the number of oriC copies per cell or measuring distances between adjacent oriC copies. Nevertheless, based on the inset in Fig. 3 , we estimated the inter-origin distance to be ~2 μm, which is only slightly larger than the distances measured in growing cultures (Fig. 1b ). Importantly, we establish that the polyploidy of B. burgdorferi cells is physiologically relevant. Fig. 3: Tick-borne B. burgdorferi cells contain multiple chromosome copies. Images of cells of strain CJW_Bb474 in the midgut of a nymphal tick 10 days after feeding drop-off. DNA was stained with Hoechst 33342. The mCherry-ParB oriC signal was amplified by staining with RFP booster. Shown are max-Z projections of a deconvolved stack of images (left) and higher-magnification views of the region indicated by the white rectangle (right). Full size image B. burgdorferi oriC copy numbers correlate with cell length In culture, strains with longer cells had higher oriC copy numbers per cell (Fig. 1b ). Correlation between oriC copy number and cell length was also apparent at the single-cell level for each strain (Supplementary Fig. 3a, b ), a scaling property that persisted after blocking cell division using the FtsI inhibitor piperacillin [51] (Fig. 4a, b ). The number of terC copies also correlated linearly with cell length (Fig. 4c, d ), as did the number of plasmid copies (Supplementary Fig. 3c, d ). We therefore approximated chromosome and plasmid densities by calculating the number of copies found in 10 μm of cell length (Fig. 1b and Supplementary Fig. 2a ). Among the B31-derived strains, those with reduced genomes (i.e., having fewer endogenous plasmids) had higher oriC densities than those with more endogenous plasmids (Fig. 1b ), suggesting that B. burgdorferi may initiate DNA replication in response to the cellular space available to be filled by the DNA. Fig. 4: B. burgdorferi chromosome copy numbers correlate with cell length. a Images of cells of strain CJW_Bb474 before (0 h) or after 24 h of exposure to piperacillin. b Correlation of oriC copy number per cell with cell length in strains CJW_Bb474 and CJW_Bb379 following the indicated durations of piperacillin treatment. r , Pearson’s correlation coefficient. c Correlations of oriC and terC copy number per cell with cell length in exponentially growing cultures of strain CJW_Bb201. r , Pearson’s correlation coefficient. d Correlations of oriC and terC copy number per cell with cell length in exponentially growing cultures of strain CJW_Bb527. r , Pearson’s correlation coefficient. e Histogram of oriC copy numbers per cell in exponentially growing cultures of strain CJW_Bb379. f Plot showing the oriC : terC ratios calculated in single cells from exponentially growing cultures of strains CJW_Bb201 and CJW_Bb527, following fluorescent spot detection. Black lines depict means ± standard deviations. Source data for panels b-f are provided as a Source Data file. The numbers ( n ) of cells analyzed and the number of replicates are provided in Supplementary Data 2 . Full size image Several lines of evidence suggest that B. burgdorferi initiates DNA replication asynchronously. First, the oriC copy number in exponentially growing B. burgdorferi cultures had a unimodal distribution (Fig. 4e ), as opposed to the expected bimodal distribution if all oriC copies would replicate at the same time. Second, at the population level, the oriC : terC ratio was ~1.2 on average, as measured both by imaging and by marker frequency analysis. Such an average oriC : terC ratio close to 1 indicates that few chromosomes are replicating at the same time, which we also confirmed at the single-cell level, as most individual cells had oriC : terC ratios smaller than 2 (Fig. 4f ). Asynchronous chromosome replication and scaling between genome copy and cell length may be a common property of polyploid bacteria, as they are also observed in cyanobacteria [52] , [53] . B. burgdorferi ParA is depleted at oriC loci We next investigated the regular spacing of chromosome copies along the cell length, which ensures near-even distribution of the chromosome to daughter cells following division at midcell. Based on the known functions of ParA and ParB in other bacteria [33] , [49] , [54] , we suspected that the B. burgdorferi parA and parB genes, which reside close to the predicted parS site (Fig. 5a ), played an important role in the regular patterning of oriC copies in B. burgdorferi . As expected, we found that the formation of mCherry-ParB foci was dependent on the presence of parS (Supplementary Fig. 1b and Supplementary Notes ). The genome-wide binding profile of mCherry-ParB, determined by ChIP-seq, revealed a broad enrichment peak that included the parS site (Fig. 6 and Supplementary Fig. 4a ). Furthermore, chromosomal replacement of parA with parA-msfgfp revealed an uneven ParA-msfGFP signal distribution along the length of the cell (Fig. 7a ). The regions of concentrated ParA-msfGFP signal alternated with regions of signal depletion that corresponded to the location of the mCherry-ParB foci in these cells, creating a banded localization pattern (Fig. 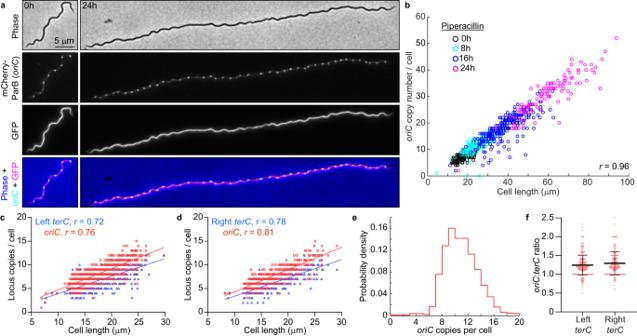Fig. 4:B. burgdorferichromosome copy numbers correlate with cell length. aImages of cells of strain CJW_Bb474 before (0 h) or after 24 h of exposure to piperacillin.bCorrelation oforiCcopy number per cell with cell length in strains CJW_Bb474 and CJW_Bb379 following the indicated durations of piperacillin treatment.r, Pearson’s correlation coefficient.cCorrelations oforiCandterCcopy number per cell with cell length in exponentially growing cultures of strain CJW_Bb201.r, Pearson’s correlation coefficient.dCorrelations oforiCandterCcopy number per cell with cell length in exponentially growing cultures of strain CJW_Bb527.r, Pearson’s correlation coefficient.eHistogram oforiCcopy numbers per cell in exponentially growing cultures of strain CJW_Bb379.fPlot showing theoriC:terCratios calculated in single cells from exponentially growing cultures of strains CJW_Bb201 and CJW_Bb527, following fluorescent spot detection. Black lines depict means ± standard deviations. Source data for panels b-f are provided as a Source Data file. The numbers (n) of cells analyzed and the number of replicates are provided in Supplementary Data2. 7a–c ). While ParA-msfGFP displayed modest accumulation between mCherry-ParB foci that were in close proximity, it accumulated prominently between mCherry-ParB foci that were farther apart (Fig. 7b, c ). This localization pattern is expected for ParA/ParB DNA partitioning systems [42] , [43] , as ParB is known to stimulate ParA depletion [55] , [56] . Fig. 5: B. burgdorferi ParB lacks the N-terminal peptide that controls ParA localization. a Schematic of the oriC -proximal chromosome region of B. burgdorferi strain B31, between nucleotides 448,705 and 459,434, showing the par genes. Features are not drawn to scale. We propose renaming the gene bb0432 of hypothetical function to parZ . b Alignment of chromosomally encoded ParB sequences from the indicated species. The first 70 positions of the alignment are shown here, while the full alignment is displayed in Supplementary Fig. 5a . Highlighted is the conserved LG(R/K)GL motif of ParB’s N-terminal ParA ATPase-stimulating peptide, which is absent from Borrelia, Streptococcus , and Staphylococcus ParB sequences. c Sequence logos for the N-terminal 20 amino acids obtained by ClustalW alignment of unique Borrelia ParZ sequences as well as unique ParB sequences from selected non-spirochete bacteria (see panel b ) or from spirochete Leptospira , Brachyspira , or Treponema genera. Only chromosome I sequences were considered for Leptospira . Boxed in are motifs similar to the conserved motif found within the N-terminal peptide of the more diverse chromosomal ParB sequences shown in ( b ). Full size image Fig. 6: B. burgdorferi ParB, ParZ, and ParA bind to the par locus. ChIP-seq profiles showing the binding of mCherry-ParB (red traces), ParZ-msfGFP (blue traces), or ParA-msfGFP (green traces) to the par region of the B. burgdorferi chromosome in the indicated strain backgrounds. Strains used, from top to bottom, are: CJW_Bb379, CJW_Bb525, CJW_Bb378, CJW_Bb524, CJW_Bb488, CJW_Bb520, CJW_Bb519, and CJW_Bb610. Genes underlining the enriched sequence reads are highlighted. aphI , kanamycin resistance gene introduced during strain generation. Full size image Fig. 7: ParZ, not ParB, controls ParA localization in B. burgdorferi . a Images of ParA-msfGFP localization in knock-in strain CJW_Bb488, which carries a full complement of par genes and thus serves as control for ParA-msfGFP localization. b Images of a cell of strain CJW_Bb538 expressing ParA-msfGFP and in which oriC copies were localized by expression of mCherry-ParB. c Fluorescence intensity profiles along the cell length for the cell shown in ( b ). d Images of ParA-msfGFP localization in knock-in strain CJW_Bb520 in which parBS is deleted. e Images of ParA-msfGFP localization in knock-in strain CJW_Bb519 in which parZ is deleted. f Images of a cell of strain CJW_Bb619 expressing ParA-msfGFP and in which parZ is deleted and oriC copies are localized by expression of mCherry-ParB. g Fluorescence intensity profiles along the cell length for the cell shown in ( f ). h Images of ParA-msfGFP localization in knock-in strain CJW_Bb610 in which parZ is missing the sequence encoding the N-terminal 20 amino acids ( parZ Δ N20 ). Full size image ParZ, not ParB, controls ParA localization in B. burgdorferi As ParB normally controls ParA localization in other bacterial ParA/ParB systems [57] , [58] , we anticipated that deletion of parB and parS ( parBS ) would disrupt the ParA banded pattern and result in a more uniform distribution. Surprisingly, deleting parBS did not eliminate the banded ParA-msfGFP localization in B. burgdorferi (Fig. 7d ). Seeking an explanation for this phenotype, we inspected the B. burgdorferi par system more closely. We noticed that B. burgdorferi ParB lacked an otherwise conserved N-terminal peptide (Fig. 5b , Supplementary Fig. 5a ), which is required for stimulation of ParA ATPase activity in other ParA/ParB systems [38] , [39] . The absence of this peptide from B. burgdorferi ParB explains its inability to control ParA localization. The ParB proteins of staphylococci and streptococci also lacked this N-terminal peptide (Fig. 5b , Supplementary Fig. 5a ). However, these bacteria also lack a ParA homolog [32] , [59] , [60] and thus do not need the ParA control function of ParB. The rest of the B. burgdorferi ParB sequence is similar to that of other chromosomal ParB proteins (Supplementary Fig. 5a ). B. burgdorferi ParA also has a typical chromosomal ParA sequence (Supplementary Fig. 5b ). Since ParB did not control ParA localization in B. burgdorferi , we hypothesized that another factor fulfilled this function. Interestingly, in B. burgdorferi , the parA and parB genes are located on the chromosome in opposite, head-to-head orientations (Fig. 5a ), instead of being joined in a two-gene operon as in many other bacteria [61] . This opposing gene organization is unique to Borreliaceae as parA and parB are organized in an operon structure in other spirochetes (Supplementary Fig. 5c ). Furthermore, parA appears to form an operon with bb0432 , a gene of hypothetical function that we propose to rename parZ (Fig. 5a ). We identified putative parAZ operons among the 29 sequenced Lyme disease Borrelia strains that we examined (Supplementary Fig. 5d ). ParZ proteins are also well conserved across the entire sequence among the larger Borreliaceae family, including relapsing fever spirochetes (Supplementary Fig. 5e ), but are not encoded by other spirochete genomes. Importantly, deletion of parZ in B. burgdorferi drastically altered the distribution of the ParA-msfGFP signal (Fig. 7e ): the banded pattern of ParA-msfGFP disappeared and the fluorescent signal became more distributed within the cell, forming only patches, likely due to the known cooperativity of ParA binding to the DNA [37] , [62] . Additionally, in the Δ parZ background, we did not detect depletion of the ParA-msfGFP signal from the vicinity of oriC , nor did we see banded accumulation of ParA-msfGFP in cellular regions located between the oriC loci (Fig. 7f, g ). We note that the ParA-msfGFP expression level was slightly increased by ~ 25% in the absence of ParZ (Supplementary Fig. 6a ). However, this small difference did not cause the loss of the ParA-msfGFP banded pattern, as the ParA-msfGFP banded pattern still required ParZ even when the fusion was overexpressed by ten-fold from a shuttle vector (Supplementary Fig. 6b, c ). Thus, ParZ regulates the subcellular localization of ParA in B. burgdorferi . In many bacteria, ParB controls ParA activity via a basic catalytic residue [38] that lies within a conserved motif, LG(R/K)GL, located in the N-terminal peptide (Fig. 5b ). Related motifs can also be found within the N-terminal peptides of chromosomal ParB sequences from spirochetes outside Borreliaceae (Fig. 5c ). Intriguingly, ParZ sequences had a similar motif in their well-conserved N-terminal peptide (Fig. 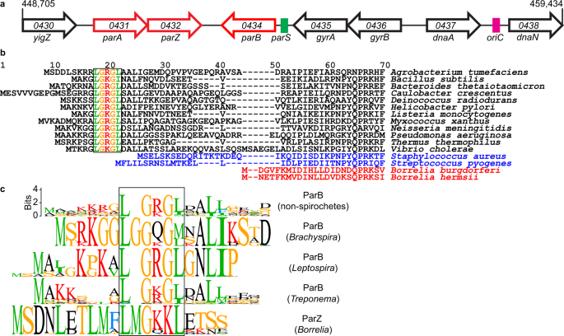Fig. 5:B. burgdorferiParB lacks the N-terminal peptide that controls ParA localization. aSchematic of theoriC-proximal chromosome region ofB. burgdorferistrain B31, between nucleotides 448,705 and 459,434, showing thepargenes. Features are not drawn to scale. We propose renaming the genebb0432of hypothetical function toparZ.bAlignment of chromosomally encoded ParB sequences from the indicated species. The first 70 positions of the alignment are shown here, while the full alignment is displayed in Supplementary Fig.5a. Highlighted is the conserved LG(R/K)GL motif of ParB’s N-terminal ParA ATPase-stimulating peptide, which is absent fromBorrelia, Streptococcus, andStaphylococcusParB sequences.cSequence logos for the N-terminal 20 amino acids obtained by ClustalW alignment of uniqueBorreliaParZ sequences as well as unique ParB sequences from selected non-spirochete bacteria (see panelb) or from spirocheteLeptospira,Brachyspira, orTreponemagenera. Only chromosome I sequences were considered forLeptospira. Boxed in are motifs similar to the conserved motif found within the N-terminal peptide of the more diverse chromosomal ParB sequences shown in (b). 5c and Supplementary Fig 5e ). Removal of this N-terminal ParZ peptide (ParZΔN20) was sufficient to disrupt ParA-msfGFP localization (Fig. 7h ), even though the peptide deletion had no apparent effect on transcription (Supplementary Fig. 6d ). Collectively, our data indicate that ParZ substitutes ParB’s function in controlling ParA localization using a similar N-terminal motif. ParZ is a novel bacterial centromere-binding protein If ParZ substitutes ParB in ParA-mediated chromosome segregation, we reasoned that ParZ must directly or indirectly bind DNA close to oriC to explain the ParA depletion at mCherry-ParB foci (Fig. 7b, c ). Indeed, chromosomal replacement of parZ with parZ-msfgfp revealed regularly spaced fluorescent foci (Fig. 8a , WT) that resembled oriC labeling by mCherry-ParB (Figs. 1 a, 8b ). The copy number and density of the ParZ-msfGFP foci were similar to those of the mCherry-ParB foci (Supplementary Fig. 6e , compare the two control strains) and the ParZ-msfGFP and mCherry-ParB foci colocalized (Fig. 8c, d ). As ParZ-msfGFP formed foci in the absence of parBS or parA (Fig. 8a ), the ParZ localization profile suggested the presence of a novel centromere-like region near oriC . Indeed, ChIP-seq experiments using ParZ-msfGFP identified a specific enrichment region that included the parAZ region (Fig. 6 ). Strikingly, this enrichment peak, which spread over a total of ~8 kilobases of DNA sequence, was adjacent to but distinct from the mCherry-ParB ChIP-seq peak (Fig. 6 , Supplementary Fig. 4a, b ). Importantly, the ParZ-msfGFP ChIP-seq peak was preserved in the Δ parBS background, as was the mCherry-ParB peak in the Δ parAZ background (Fig. 6 ), in agreement with our microscopy observations (Fig. 8a, b ). If ParZ binds within its own gene, it predicts that ectopic expression of parZ on a shuttle vector will increase the number of fluorescent ParZ-msfGFP puncta given that the shuttle vector is in ~5-fold higher copy number than the chromosome [22] , [23] , [63] . This is indeed what we observed (Supplementary Fig. 4f, g ). Additionally, the presence of an empty shuttle vector in the strain expressing ParZ-msfGFP from the endogenous locus did not cause an increase in the number of ParZ-msfGFP puncta (Supplementary Fig. 4g ). Furthermore, ChIP-seq in strain CJW_Bb101 carrying parZ-msfgfp on the shuttle vector confirmed binding of ParZ within the shuttle vector sequence (Supplementary Fig. 4c, d ), in addition to the native parZ region on the chromosome (Supplementary Fig. 4e ). Altogether, these observations suggest that ParZ binds within its own gene. Fig. 8: ParZ is a novel bacterial centromere-binding protein that contributes to oriC segregation. a Images of ParZ-msfGFP signal in strains carrying the full complement of B. burgdorferi par genes (WT) or lacking the par genes and/or parS sequence as indicated. DNA was stained with Hoechst 33342. CJW_Bb strain numbers are listed on the phase-contrast images. b Images of mCherry-ParB signal in strains carrying the full complement of par genes (WT) or lacking the parAZ operon, as indicated. DNA was stained with Hoechst 33342. CJW_Bb strain numbers are listed on the phase contrast images. c Images of strain CJW_Bb403 showing colocalization of ParZ-msfGFP and mCherry-ParB signals. d Fluorescence intensity profile along the cell length for the cell shown in ( c ). e Histograms showing the distributions of deviations from uniform spacing (DUS, see methods) of oriC spots in control strains expressing mCherry-ParB (strain CJW_Bb379) or ParZ-msfGFP (strain CJW_Bb378) to label oriC . Also shown in gray are DUS values obtained by simulating a random redistribution of oriC loci in the analyzed cells of strain CJW_Bb379 (see methods). f Histograms comparing DUS distributions of ParZ-msfGFP-labeled oriC foci in control (CJW_Bb378), Δ parBS (CJW_Bb524), Δ parA (CJW_Bb490), and Δ parA Δ parBS (CJW_Bb616) strains. g Histograms comparing DUS distributions of mCherry-ParB-labeled oriC foci in control (CJW_Bb379), Δ parAZ (CJW_Bb525), and Δ parZ (CJW_Bb626) strains. Source data for panels (e–g) are provided as a Source Data file. The numbers ( n ) of cells analyzed and the number of replicates are provided in Supplementary Data 2 . Full size image In traditional ParA/ParB systems, ParB bound to parS and adjacent sequences controls ParA localization by transiently interacting with ParA [33] . If ParZ works via a similar mechanism in B. burgdorferi , it predicts a transient interaction between ParZ and ParA. ChIP-seq experiments verified this prediction as the ParA-msfGFP enrichment peak was at the same location as the ParZ-msfGFP peak, albeit at a lower level consistent with a transient interaction (Fig. 6 and Supplementary Fig. 4a ). We also observed low-level, non-uniform mapping of ParA-msfGFP ChIP-seq reads to B. burgdorferi ’s endogenous plasmids (Supplementary Fig. 4a, h ). Since free GFP, ParZ-msfGFP, ParA-msfGFP, and mCherry-ParB pulldowns generated almost identical traces in this region (Supplementary Fig. 4h ), we believe these traces represent non-specific landscape binding. ParA-msfGFP binding to the par locus, while reduced in the parBS mutant, was nevertheless still present (Fig. 6 ), indicating that ParA recruitment to the par locus did not require parBS . In contrast, ParA-msfGFP recruitment to the par locus required ParZ and, more specifically, its N-terminal peptide (Fig. 6 ). These results indicate that ParZ is a newly identified centromeric protein, which, similarly to ParB in other bacteria [38] , [39] , uses its N-terminal peptide to regulate ParA localization. ParA, ParB, and ParZ jointly control chromosomal oriC spacing Given that ParZ, and not ParB, controls ParA in B. burgdorferi , we investigated the role of each Par protein in oriC segregation using a comprehensive set of par gene deletion mutants. In the absence of an appropriate setup for live-cell timelapse imaging of B. burgdorferi , we analyzed static snapshots of exponentially growing populations of cells. Visual inspection of the control strains that express mCherry-ParB or ParZ-msfGFP to label oriC revealed a near-equidistant spacing of oriC copies along the cell length (Fig. 8a, b , WT). For quantification, we calculated how much the ori C distribution in each cell of a population deviates from uniform spacing (see methods). This metric, referred to as d eviation from u niform s pacing (or DUS), gives a value of 0 when a cell displays a perfectly equidistant distribution of oriC copies. In contrast, a random intracellular distribution of oriC copies yields an average DUS value of 0.7 (Fig. 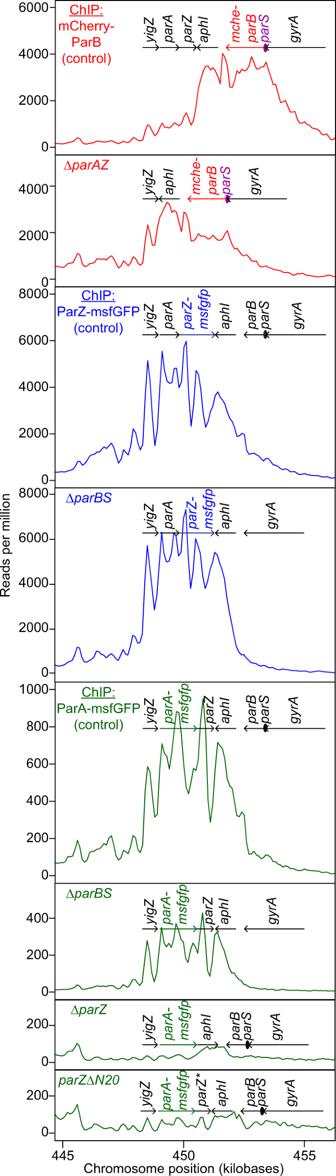Fig. 6:B. burgdorferiParB, ParZ, and ParA bind to theparlocus. ChIP-seq profiles showing the binding of mCherry-ParB (red traces), ParZ-msfGFP (blue traces), or ParA-msfGFP (green traces) to theparregion of theB. burgdorferichromosome in the indicated strain backgrounds. Strains used, from top to bottom, are: CJW_Bb379, CJW_Bb525, CJW_Bb378, CJW_Bb524, CJW_Bb488, CJW_Bb520, CJW_Bb519, and CJW_Bb610. Genes underlining the enriched sequence reads are highlighted.aphI, kanamycin resistance gene introduced during strain generation. 8e and see methods). Control strains, which have a complete set of parA, parZ, and parB genes, had very similar DUS distributions centered around ~0.2 (Fig. 8e ), indicating near-equidistant spacing. Deletion of parBS reduced the number of oriC foci (Supplementary Fig. 6e ) but had little impact on the regularity of oriC spacing (Fig. 8a ). This was reflected in the DUS distribution, which displayed only a slight shift towards larger values relative to the control strains (Fig. 8f ). In contrast, deletion of parA or parAZ resulted in some disruption of oriC spacing (Fig. 8a, b ). This was quantitatively reflected in larger, rightward shifts of DUS distributions (Fig. 8f, g ). Surprisingly, deletion of parZ alone caused a larger disruption of oriC spacing than the removal of parA or parAZ (Fig. 8g ). It may suggest that a dysregulated ParA activity is more detrimental than no ParA activity at all. The combination of Δ parA and Δ parBS in strain CJW_Bb616 caused the strongest oriC spacing defect. This defect manifested as multiple oriC foci clustered in one or several short cell segments flanked by large cellular spaces containing DNA devoid of oriC spots (Fig. 8a ). This striking phenotype resulted in the largest DUS distribution shift towards higher values (Fig. 8f, g ). Furthermore, the severe oriC segregation defect seen in the Δ parA Δ parBS double mutant was accompanied by a large increase in the frequency of cells that lacked oriC foci, from <0.3% in control strains to 3.5% in the Δ parA Δ parBS double mutant (Supplementary Fig. 6e ). Collectively, our findings indicate that parA/parZ and parB/parS jointly control oriC segregation in B. burgdorferi , with parA/parZ playing a more prominent role. ParB recruits SMC to the chromosomal replication origins Despite having lost its ability to control ParA, B. burgdorferi ParB still participates in oriC segregation (Fig. 8f ). Therefore, we investigated whether ParB achieves this function via interaction with another protein. In other bacteria, ParB recruits structural maintenance of the chromosome (SMC) complexes to the oriC region [64] , [65] , [66] . The recruitment of SMC to oriC and subsequent organization of the oriC region have been shown to facilitate oriC segregation in Caulobacter crescentus and Bacillus subtilis [64] , [65] , [66] , [67] , [68] , [69] , [70] . While lacking the ParA control motif, the B. burgdorferi ParB protein has retained a predicted SMC-binding region located within the N-terminal domain of ParB [66] (Supplementary Fig. 5a ). B. burgdorferi also encodes a homolog of SMC at locus bb0045 . We therefore replaced smc with an mcherry-smc fusion both in the wild-type background and in a strain that expresses ParZ-msfGFP to visualize the oriC region. mCherry-SMC had no detectable effect on oriC copy number (Supplementary Fig. 6e ) and formed fluorescent foci that colocalized with some, though not all, ParZ-msfGFP-decorated oriC loci (Fig. 9a, b ). Consistent with this colocalization, ChIP-seq experiments revealed enrichment of mCherry-SMC at the par locus, centered around the parS site, which is consistent with its recruitment by ParB (Fig. 9c ). Deletion of parBS abrogated the formation of clear mCherry-SMC puncta (Fig. 9a, b ), resulting in a loss of colocalization between mCherry-SMC and ParZ-msfGFP-decorated oriC loci. Finally, the Δ smc mutation caused a similar reduction in oriC copy number and density as Δ parBS (Supplementary Fig. 6e ) and mildly disrupted oriC spacing (Fig. 9d, e ). These results support the idea that ParB recruits SMC near oriC , and that this interaction plays a supporting role in oriC segregation in B. burgdorferi . The synergy between the ParA/ParZ and ParB/SMC systems in oriC partitioning was substantiated by the presence of a synthetic growth defect when both systems were defective (Δ parAZBS background), as measured both in semisolid plates and liquid cultures (Supplementary Fig. 6g, h ). Fig. 9: SMC is recruited to the oriC region by ParB and mildly contributes to regular oriC spacing. a Images of cells expressing ParZ-msfGFP (to label oriC ) and mCherry-SMC in control (CJW_Bb602, carrying the full complement of par genes) and Δ parBS (CJW_Bb615) strains. b Fluorescence intensity profiles along the cell length for the cells shown in ( a ). c ChIP-seq profile showing the binding of mCherry-SMC to the par locus in strain CJW_Bb601. Genes underlining the enriched sequence reads are highlighted. d Images of cells showing oriC localization in Δ smc strains in which the oriC is labeled with either ParZ-msfGFP (CJW_Bb603) or mCherry-ParB (CJW_Bb604). Hoechst 33342 was used to stain the DNA. An overlay is also shown. e Histograms showing DUS of oriC spots in cells of control and Δ smc strains in which oriC was labeled with either ParZ-msfGFP (control, CJW_Bb378; Δ smc , CJW_Bb603) or mCherry-ParB (control, CJW_Bb379; Δ smc , CJW_Bb604). Also shown is the DUS histogram for the Δ parBS strain CJW_Bb524. Source data are provided as a Source Data file. The numbers ( n ) of cells analyzed and the number of replicates are provided in Supplementary Data 2 . Full size image Our live-cell imaging provides definite proof that the B. burgdorferi chromosome and plasmids exist in multiple copies during the growth phase of this spirochete (Figs. 1 , 2 , Supplementary Figs. 1c , 2 ). This dispels the notion that Lyme disease agents such as B. burgdorferi differ in ploidy from the relapsing fever agent Borrelia hermsii , which was shown to have multiple genome copies per cell using biochemical population-level measurements [24] , [71] . We note that fragmentation of DNA staining had been reported in air-dried B. hermsii and B. burgdorferi cells [24] , [72] . However, comparison with biochemical quantification of genome copy numbers [24] demonstrate that this approach is probably not reliable to assess ploidy. This is not surprising given that cellular desiccation is well known to result in double-stranded DNA breaks. In contrast, our imaging results using live B. burgdorferi cells are in good agreement with qPCR analysis (Fig. 1f-g and Supplementary Fig. 1h ). Interestingly, qPCR experiments have also demonstrated the polyploid nature of the syphilis spirochete Treponema pallidum [73] . Thus, polyploidy may reflect a general property of spirochetes. Polyploidy may be advantageous under stress. For instance, the presence of multiple genome copies has been shown to increase resistance to DNA damage in cyanobacteria [74] , presumably by facilitating DNA recombination and repair. Polyploid cyanobacteria can also recover from infection by lytic phages as long as not all genome copies are degraded prior to phage inactivation [75] . In the context of a pathogen like B. burgdorferi , polyploidy may facilitate persistence in the vertebrate host. Modeling studies have predicted that antigenic variation systems facilitate longer survival of pathogens in immunocompetent hosts when they are present in multiple genomic copies than when encoded on a single-copy genome [71] . The plasmid lp28-1 contains an antigen variation system [76] . Its presence in multiple copies (Fig. 2 ) may further help this spirochete evade the host antibody response. B. burgdorferi polyploidy also has practical implications, one being B. burgdorferi load assessment in animal tissues by qPCR which often assumes that one genome copy represents one bacterial cell [19] . Actual tissue bacterial loads could be ~10-fold lower. In this study, we also demonstrated the regular subcellular distribution of both chromosome and plasmid copies (Figs. 1 a, 2 a, 8e and Supplementary Fig. 1c ). In the context of symmetric division (i.e., at midcell) [28] , such a regular linear distribution of a multicopy genome ensures that each daughter cell inherits near-equal copies of the genome, as in cyanobacteria [52] , [53] . Indeed, severe disruption of near-uniform distribution of the B. burgdorferi chromosome in the Δ parA Δ parBS mutant (Fig. 8a,f ) was accompanied by chromosome inheritance defects (Supplementary Fig. 6e ). Regular genome patterning also implies the existence of active segregation mechanisms. For the B. burgdorferi plasmids, the conserved plasmid maintenance loci [31] are likely responsible for their observed subcellular distribution. For bacterial chromosomes, segregation of the oriC regions generally involves ParB-dependent control of ParA activity. Unexpectedly, we found that in B. burgdorferi , and presumably other Borrelia species, the localization of ParA is instead primarily controlled by a novel centromere-binding protein, which we named ParZ (Figs. 5 – 8 , Supplementary Figs. 4 – 6 ). Control of ParA by factors other than ParB has previously been documented in Myxococcus xanthus , where the CTPase PadC recruits ParA to subpolar bactofilin structures [35] , [77] , although M. xanthus ParB retains its ParA-stimulating peptide (Fig. 5b ) and the ability to control ParA localization [78] . In B. burgdorferi , we envision that the ParA/ParZ system harnesses forces within the cell to drive segregation of the oriC loci, similarly to how the ParA/ParB system drives patterning of multicopy plasmids [33] , [42] , [49] . ParZ displays several other properties reminiscent of ParB. Like ParB, ParZ appears to spread on the DNA around its cognate centromeric site, occupying several kilobases of DNA sequence (Fig. 6 ). Additionally, ParZ binding to the DNA is not uniformly distributed; rather, it displays several peaks and valleys, which was also observed in the case of ParB [79] , [80] . This broad distribution of ParZ binding likely increases the probability of interaction with ParA. Future investigation will be required to uncover the mechanisms underlying ParZ spreading, including whether it shares any mechanistic similarities with ParB, such as CTPase (or other NTPase) activity, clamp formation, and lateral sliding along the DNA [33] , [34] , [35] , [81] . In B. burgdorferi , interestingly, ParB spread from the parS site appears skewed in one direction that matches that of the transcription of the bound genes (Fig. 6 ). In turn, binding of ParB to the DNA decreases when the bound genes become convergently transcribed with the direction of ParB spread (Fig. 6 and Supplementary Fig. 4b ). We observed a similar behavior for ParZ in several genetic backgrounds (Fig. 6 and Supplementary Fig. 4b, d , e). This raises the possibility that active transcription promotes the spread of ParB and possibly ParZ away from the loading site when the direction of spread and transcription are the same and limits the spread when transcription and spread occur in opposite directions. A similar inference can be gleamed from ChIP-seq traces of ParB binding to the DNA in Corynebacterium glutamicum [82] . Additionally, transcription of underlying genes was invoked to explain asymmetric spread of ParB onto parS -proximal DNA sequences in C. crescentus [79] . While ParB lost its ability to control ParA localization in B. burgdorferi , it retained its role in recruiting SMC to oriC (Fig. 9 ), thereby contributing to oriC partitioning, though to a lesser degree than the ParA/ParZ system (Fig. 8f ). SMC, possibly through the organization of the oriC region [69] , also promotes oriC segregation. This is evident from the similar oriC segregation defects displayed by the Δ parBS and Δ smc mutants (Fig. 9e ). The ParB/SMC system, as well as ParA, may also be involved in initiation of DNA replication [83] , as several par and smc mutants that we characterized have decreased oriC copy numbers during exponential growth in culture (Supplementary Fig. 6e ). During the evolution of Borreliaceae, ParB retained a SMC loading function but remarkably transferred its ParA-regulating function to a new player. How could it have happened? BLAST searches allowed us to identify distant homologs of ParZ among the Firmicutes and Fusobacteria (Supplementary Fig. 7 ). The Streptococcus , Staphylococcus , Enterococcus , and Bacillus genera are particularly well represented among the Firmicutes hits (Supplementary Fig. 7 ). These ParZ-like proteins contain only short regions of homology with the Borreliaceae ParZ proteins and do not include the ParB-like N-terminal peptide. More intriguing though is that a subset of these ParZ-like proteins are encoded by phages (Supplementary Fig. 7 ). It is tantalizing to speculate acquisition of parZ from a phage infection of the spirochete ancestor of the Borreliaceae. In fact, Borrelia genomes carry extensive evidence of infection by phages, including those related to known streptococcal phages [18] . Phage insertion into the parB gene may have fused the sequence encoding the N-terminal, ParA-controlling peptide of ParB to a phage-encoded protein that binds its own DNA sequence. Subsequent genetic drift of the phage-disrupted spirochete genome may have resulted in inversion of the orientation of the parB gene and loss of the remaining phage sequence, generating the current locus structure. While this evolutionary scenario remains speculative, our findings highlight the plasticity and evolvability of microbial genomes, even in the context of fundamental cellular functions such as genome partitioning. Understanding basic biological functions in non-model species is important, particularly in bacterial pathogens where divergent regulatory mechanisms of essential bacterial functions may provide new targets for specific therapeutic intervention. Bacterial strains and growth conditions The following Escherichia coli cloning strains were used to generate, maintain, and grow the various plasmids used in this study: DH5α (Promega), NEB 5-alpha and NEB 5-alpha F’ l q (New England Biolabs), and XL10-Gold (Agilent). The strains were grown on Luria Bertani agar plates incubated at 30 °C or in Super Broth (35 g/L bacto-tryptone, 20 g/L yeast extract, 5 g/L NaCl, and 6 mM NaOH) liquid medium with shaking at 30 °C. Antibiotics were used at the following concentrations: kanamycin at 50 μg/mL, gentamicin at 15 to 20 μg/mL, spectinomycin or streptomycin at 50 μg/mL, rifampin at 25 μg/mL in liquid culture or 50 μg/mL in plates, and hygromycin B at 100 to 200 μg/mL. B. burgdorferi strains and their generation are detailed in Supplementary Data 1 , Worksheet 1. Requests for the B. burgdorferi strains generated in this study should be directed to Christine Jacobs-Wagner. These strains were grown in complete Barbour-Stoenner-Kelly (BSK)-II liquid medium in humidified incubators at 34 °C under 5% CO 2 atmosphere [6] , [10] , [11] . Complete BSK-II medium contained 50 g/L bovine serum albumin (Millipore #810036), 9.7 g/L CMRL-1066 (US Biological #C5900-01), 5 g/L Neopeptone (Difco #211681), 2 g/L Yeastolate (Difco #255772), 6 g/L HEPES (Millipore #391338), 5 g/L glucose (Sigma-Aldrich #G7021), 2.2 g/L sodium bicarbonate (Sigma-Aldrich #S5761), 0.8 g/L sodium pyruvate (Sigma-Aldrich #P5280), 0.7 g/L sodium citrate (Fisher Scientific #BP327), 0.4 g/L N -acetylglucosamine (Sigma-Aldrich, #A3286), 60 mL/L heat-inactivated rabbit serum (Gibco #16120), and had a pH of 7.60. Complete BSK-H media was acquired from Sigma-Aldrich (#B8291). Tubes contained 6 to 7 mL or 13 to 15 mL culture depending on the tube size used (8-mL volume, Falcon, #352027, or 16-mL volume, Falcon, #352025) and were kept tightly closed. Any larger volume vessels were kept loosely capped in the incubator. BSK-1.5 medium for plating was previously described [12] , [84] , [85] and contained 69.4 g/L bovine serum albumin, 12.7 g/L CMRL-1066, 6.9 g/L Neopeptone, 3.5 g/L Yeastolate, 8.3 g/L HEPES, 6.9 g/L glucose, 6.4 g/L sodium bicarbonate, 1.1 g/L sodium pyruvate, 1.0 g/L sodium citrate, 0.6 g/L N -acetylglucosamine, and 40 mL/L heat-inactivated rabbit serum, and had a pH of 7.50. Selection antibiotics were used at the following final concentrations in both liquid cultures and plates: kanamycin at 200 μg/mL [86] , gentamicin at 40 μg/mL [87] , streptomycin at 100 μg/mL [88] , hygromycin B at 300 μg/mL [85] , [89] and blasticidin S at 10 μg/mL [89] . Piperacillin was used at a final concentration of 10 ng/mL. Unless otherwise indicated, all cultures were maintained in exponential growth by diluting the cultures into fresh medium before reaching ~5 × 10 7 cells/mL. Semisolid BSK-agarose plating medium [85] contained 2 parts of 1.7% agarose solution in water and 3 parts BSK-1.5 medium containing appropriate amounts of selective antibiotics, as needed, to yield in the final plating mix the concentrations listed above. Each plate was seeded with a maximum of 1 mL B. burgdorferi culture. The agarose, melted and maintained at 55 °C, and the BSK-1.5 medium, briefly pre-equilibrated at 55 °C, were mixed and then 25 mL were poured into each B. burgdorferi -seeded plate. The plates were swirled gently to mix, allowed to solidify at room temperature (RT) in a biosafety cabinet for ~ 30 min, then transferred to a humidified CO 2 incubator and incubated between 10 days and 3 weeks. Genetic manipulations All plasmids (Supplementary Data 1 , Worksheet 2) were generated using standard molecular biology techniques that included ligation of restriction endonuclease-digested plasmids and PCR products, Gibson assembly [90] of DpnI-digested PCR products using New England Biolabs’ platform, or site-directed mutagenesis using the Agilent Quick Change Lightning Site-Directed Mutagenesis kit. Sequences of the oligonucleotide primers used in the course of plasmid generation are provided in Supplementary Data 1 , Worksheet 3. The plasmids, for which relevant sequences were confirmed by Sanger DNA sequencing at Quintara Biosciences, were introduced into E. coli host strains by heat shock or electroporation and were archived as E. coli strains. Minipreps were done with Zymo Research Zippy plasmid miniprep kit. When requesting any plasmid, we urge the requestor to provide us with the E. coli CJW strain number listed in Supplementary Data 1 , Worksheet 2, in addition to the name of the plasmid. Large amounts of plasmid DNA were isolated from saturated 50 mL Super Broth E. coli cultures using the Qiagen Plasmid Plus Midi kit with the final elution performed in water. E. coli / B. burgdorferi shuttle vectors (25 to 50 μg) were electroporated into 50-100 μL volumes of B. burgdorferi competent cells, which were prepared as previously described [91] by various concentrations and washing steps using electroporation solution (93.1 g/L sucrose, American Bioanalytical #AB01900, 150 mL/L glycerol, American Bioanalytical #AB00751) and 10 min centrifugation steps at 4 °C and 10,000 × g in the FX6100 rotor of a Beckman Coulter Allegra X-14R centrifuge. Suicide vectors (50–75 μg) were linearized with the restriction endonucleases indicated in Supplementary Data 1 , Worksheet 1, ethanol precipitated [92] , resuspended in 25 μL water, then electroporated into 100 μL aliquots of B. burgdorferi competent cells. Electroporation was done at 2.5 kV, 25 μF, and 200 Ω [12] , [84] in a 2 mm-gap cuvette. The electroporated cells were immediately recovered in 6 mL BSK-II medium, and incubated overnight at 34 °C, after which selection in liquid culture and in semisolid BSK-agarose plates was performed. When needed, non-clonal, liquid-selected populations of transformants were plated in semisolid BSK-agarose for clone isolation. For each B31-derived clone, we confirmed the endogenous plasmid complement by multiplex PCR [93] . Plasmid complement was not determined for clones derived from strains other than B31 due to the absence of a complete, standardized PCR primer set for those strains. To confirm the correct homologous recombination of suicide vectors, total genomic DNA was isolated from the B. burgdorferi clones using the Qiagen DNeasy Blood & Tissue Kit, and diagnostic PCR was performed to confirm insertion or deletion within the targeted locus, as well as correct recombination of the flanking sequences. The genetic manipulations of the chromosome at the par and smc loci are depicted schematically in Supplementary Fig. 8 . Insertion of parS P1 cassettes at the phoU , uvrC , and lptD loci occurred in intergenic regions between two convergently transcribed genes. The same strategy was used to insert the parS P1 cassette in B. burgdorferi plasmids. For the cp32 plasmids, the parS P1 cassette was inserted into the transposon sequence in transposon mutant backgrounds for which the transposon was mapped to have inserted in an intergenic region flanked by convergently transcribed genes [30] . As a result, the likelihood of coding sequence or promoter disruption by the genetic changes was minimized. An exception is lp25, where the cassette was inserted in the scar generated upon deletion of the nonessential gene bbe02 . Mouse-tick transmission studies Ethics statement All animal work was performed according to the guidelines of the National Institutes of Health, Public Health Service Policy on Humane Care and Use of Laboratory Animals and the United States Institute of Laboratory Animal Resources, National Research Council, Guide for the Care and Use of Laboratory Animals. Protocols were approved by the Rocky Mountain Laboratories, NIAID, NIH Animal Care and Use Committee. The Rocky Mountain Laboratories are accredited by the International Association for Assessment and Accreditation of Laboratory Animal Care (AAALAC). All efforts to minimize animal suffering were made. Experimental mouse-tick infection studies Mouse ( Mus musculus ) infections were conducted with 4-8 weeks-old female RML mice, an outbred strain of Swiss-Webster mice reared at the Rocky Mountain Laboratories breeding facility. Mice were housed at an ambient temperature between 20.6 and 23.9 °C, ambient humidity of 50%±10%, and under a 12 h ON / 12 h OFF light cycle. Five mice per strain were inoculated intraperitoneally (4 ×10 4 spirochetes) and subcutaneously (1 × 10 4 spirochetes), with the number of injected spirochetes pre-determined by Petroff-Hausser counting. Mouse infection was confirmed 3 weeks post-injection by isolation of B. burgdorferi from ear biopsies in BSK-II medium containing appropriate antibiotics. Larval Ixodes scapularis were purchased from Oklahoma State University. I. scapularis were maintained between feeds at ambient light and temperature in bell jars over potassium sulfate-saturated water. Approximately 100 naïve I. scapularis larvae were fed to repletion per infected mouse. Acquisition and retention of B. burgdorferi by larval ticks was assessed 1 week after drop-off, and spirochete load was determined through mechanical disruption and plating. Two naïve mice per strain were fed upon by 15-20 infected I. scapularis nymphs. The number of B. burgdorferi in nymphs was assessed prior to feeding and 10 days after drop-off through mechanical disruption and plating. Mouse infection was confirmed 5 weeks post-nymphal tick feeding by isolation of B. burgdorferi from ear biopsies in BSK-II medium containing appropriate antibiotics. Tick midgut cryopreservation Tick midguts were dissected and fixed on ice using 4% formaldehyde solution in phosphate buffered saline (PBS), washed thrice for 5 min with cold PBS, infiltrated with 15% sucrose in PBS at 4 °C, then with 30% sucrose in PBS at 4 °C, then with a 1:1 mix of 30% sucrose in PBS and Optimal Cutting Temperature (OCT) compound (Tissue-Tek), and finally with pure OCT compound. The tissue was then frozen in OCT compound using liquid-nitrogen-cooled isopentane, then stored at −80 °C and shipped on dry ice. Thin, 10-μm sections were cut using a cryostat. Microscopy B. burgdorferi culture density was measured by dilution of a culture in a C-Chip disposable hemocytometer (INCYTO) and direct counting of the cells under darkfield illumination obtained using a Nikon Eclipse E600 microscope equipped with a 40×0.55 numerical aperture (NA) Ph2 phase-contrast air objective and darkfield condenser optics. 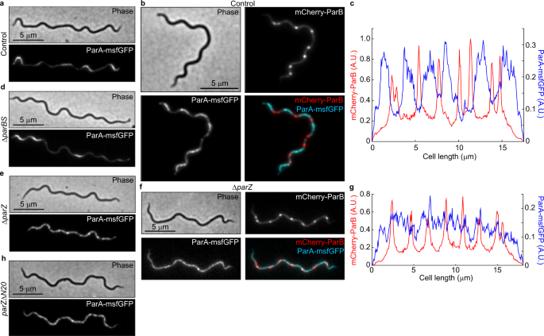Fig. 7: ParZ, not ParB, controls ParA localization inB. burgdorferi. aImages of ParA-msfGFP localization in knock-in strain CJW_Bb488, which carries a full complement ofpargenes and thus serves as control for ParA-msfGFP localization.bImages of a cell of strain CJW_Bb538 expressing ParA-msfGFP and in whichoriCcopies were localized by expression of mCherry-ParB.cFluorescence intensity profiles along the cell length for the cell shown in (b).dImages of ParA-msfGFP localization in knock-in strain CJW_Bb520 in whichparBSis deleted.eImages of ParA-msfGFP localization in knock-in strain CJW_Bb519 in whichparZis deleted.fImages of a cell of strain CJW_Bb619 expressing ParA-msfGFP and in whichparZis deleted andoriCcopies are localized by expression of mCherry-ParB.gFluorescence intensity profiles along the cell length for the cell shown in (f).hImages of ParA-msfGFP localization in knock-in strain CJW_Bb610 in whichparZis missing the sequence encoding the N-terminal 20 amino acids (parZΔN20). For fluorescence microscopy imaging, BSK-II-grown B. burgdorferi strains were spotted onto a 2% agarose-PBS pad [28] , [94] , covered with a no. 1.5 coverslip, then imaged using Nikon Eclipse Ti microscopes equipped with 100X Plan Apo 1.45 NA phase-contrast oil objectives, Hamamatsu Orca-Flash4.0 V2 CMOS cameras, and either a Sola LE light source or a Spectra X Light engine (Lumencor). The microscopes were controlled by Nikon Elements software. The following Chroma filter cubes were used to acquire the fluorescence images: DAPI, excitation ET395/25x, dichroic T425lpxr, emission ET460/50 m; GFP: excitation ET470/40x, dichroic T495lpxr, emission ET525/50 m; mCherry/TexasRed, excitation ET560/40x, dichroic T585lpxr, emission ET630/75 m. DNA staining was obtained by incubating the culture for 15 min with Hoechst 33342 (Molecular Probes) at a final concentration of 1 μg/mL. Tick midgut sections (see above) were processed as follows. The slides supporting the sections were brought up to RT, washed thrice with PBS, permeabilized for 30 min at RT using 0.2% Triton X-100 in PBS, blocked for 30 min at RT using 5% bovine serum albumin (BSA) (w/v) in PBS, 0.1% Tween-20, stained with RFP-Booster ATTO594 (ChromoTek) diluted 1:200 in blocking buffer (see above), washed thrice with PBS for 5 min each, and stained with Hoechst 33342 1:1000 in PBS for 10 min. The stained sections were mounted in PBS under a No 1.5 coverslip and were imaged on an OMX BLAZE microscope system (GE). Images in the DAPI, GFP, and mCherry channels were acquired at 100 nm z intervals. The image stacks were then deconvolved and registered using the Softworks software. Image analysis Cell outlines were generated using phase-contrast images and the Oufti analysis software package [95] , with the following parameters: Edgemode, LOG; Dilate, 2; openNum, 3; InvertImage, 0; ThreshFactorM, 0.985; ThreshMinLevel, 0; EdgeSigmaL, 1; LogThresh, 0. Cell outlines were curated as follows: (i) outlines of cell debris were manually removed; (ii) outlines of cells that curled on themselves, crossed other cells, or were partially outside the field of view were also manually removed; (iii) partial outlines of cells were manually extended when feasible; (iv) outlines were manually added in some cases where automated outline generation failed; and (v) outlines were manually split for cells displaying clear phase profile dips around midcell, which indicated that the cytoplasmic cylinders of the daughter cells had separated yet remained linked by an outer membrane bridge [28] . This was confirmed by visual inspection of the fluorescence signal(s), as phase profile midcell dips often corresponded to a dip in the fluorescence signal. For this reason, throughout the manuscript, the term cell refers to an individual cytoplasmic cylinder. Lastly, the “Refine All” function of the Oufti software was ran, a final curation removed improper outlines, and the fluorescence signal was added to the cell outline file in Oufti. For signal quantification and intensity profile generation, we used the Oufti background fluorescence subtraction and intensity profile generation features. Image visualization was done using FiJi software [96] , GraphPad Prim 9.3.1 software, and Adobe Illustrator 2023. To detect fluorescent spots, the Modified_Find_Irregular_Spots.m MATLAB function [97] was used, with the following parameters: fitRadius: 5, edgeDist: 2.5, centerDist: 1; peakRadius: 3; shellThickness: 1; quantileThreshold: 0.3. The value of the intensityRatioThreshold parameter was determined individually for each microscopy experiment and fluorescence channel. For each intensityRatioThreshold value empirically tested, visual inspection of the accuracy of spot detection was performed on a subset of the cells using the VisualizeSpotDetection.m function. Once an appropriate intensityRatioThreshold value was identified, all the cell outlines were visually inspected and the ones that displayed under- or over-detection of spots were manually removed, yielding a curated cell list. Then, spots were identified and added to this final cell list using the add_spots_to_cellList.m routine, while the data was exported into a table format using export_to_table.m and extract_field.m routines. A summary of the imaging experiments is provided in Supplementary Data 2 , Worksheet 1. Each experimental sample was given a unique identifier. Thus, replicates of a given strain will have different identifiers. This summary includes the following information for each experiment: strain name, replicate number, relevant treatments, culture density at the time of image acquisition, number of cells, and intensityRatioThreshold values used to detect the fluorescent spots. The oriC : terC ratio was calculated from microscopy data as follows: (i) the oriC and terC copy number per cell was plotted as a function of cell length in GraphPad Prism; (ii) a linear fit of the data was performed, and the slope of each fit was extracted; and (iii) the slope of the oriC fit was divided by the slope of the terC fit. To quantify the extent to which the distribution of the oriC spots along the length of the cell deviates from an equidistant distribution, we performed the following analysis steps for each cell. First, we measured all distances between adjacent oriC spots, or DM (for distance measured). A cell with n spots will generate n −1 DM values. Next, in silico and for each cell individually, we equidistantly redistributed the oriC spots within the length of that cell, using the calculate_distance_ratio.m routine. This analysis assumes that each oriC spot is separated from the adjacent oriC spot or from the adjacent cell end (for the first and last oriC spot in a given cell, respectively) by the same distance. In this scenario, the distance DE between adjacent, equidistantly redistributed spots for a given cell is: 
    DE=L/n+1
 (1) where L is the length of the cell and n is the number of oriC spots in the cell. Then, for each pair of adjacent oriC spots, we calculated a distance ratio, DR, defined as the ratio of the measured distance between two adjacent spots and the value this distance would have if all the spots in the cell were equidistantly spaced. DR_i=DM_i/DE
 (2) Therefore, for a perfectly equidistant distribution of oriC spots, all distance ratios are exactly 1. Finally, to assess how the oriC spots of a given cell deviate from equidistant spacing, we calculated a deviation from uniform spacing (or DUS) metric defined as the mean per cell of the absolute values of the deviation of the DR values from 1: 
    DUS= ∑_i=1^n-1|DR_i-1|/n-1
 (3) Please note that in a cell with n spots, there will be n −1 distances between adjacent spots. The data shown in Figs. 8 e–g and 6e show the distribution of DUS values within the population of cells of the indicated strains. We also simulated a random distribution of oriC copies inside the cells using the simulate_distance_ratio.m routine. For each analyzed cell (see above), this routine randomly redistributes each cell’s oriC copies along the length of that cell, then extracts the distances between adjacent randomly redistributed oriC spots and calculates the DR and DUS values as above. Sample growth for next-generation sequencing A summary of the ChIP-seq samples analyzed and reported in this study is given in Supplementary Data 2 , Worksheet 2. For each strain and replicate, we provide information on culture growth conditions, inoculation and harvesting dates, and harvesting culture densities. The samples were prepared as follows. Exponentially growing B. burgdorferi strains were used to inoculate 250 mL BSK-II cultures. After two or three days of growth the cultures were fixed by addition of 95 mL 37% formaldehyde (Sigma-Aldrich #F8775) followed by incubation with rocking for 30 min at RT. Formaldehyde was then quenched by addition of 18 mL of 2.5 M glycine followed by incubation with rocking for 5 min at RT. The samples were chilled on ice for 10 min, transferred to conical centrifuge tubes and pelleted at 4 °C using a 30 min, 4300 × g spin in an Allegra X-14R centrifuge (Beckman Coulter) equipped with a swinging bucket SX4750 rotor. The pellet was resuspended in 30 mL ice-cold HN buffer (50 mM NaCl, 10 mM HEPES, pH 8.0) [98] , then pelleted at 4 °C and 10,000 × g for 10 min in a fixed angle FX6100 rotor. The pellet was resuspended in 1.5 mL final cold HN buffer and pelleted once more at 4 °C and 10,000 × g for 10 min. Finally, the pellet was resuspended in 500 μL ice-cold ChIP buffer A (12.5 mM Tris, 12.5 mM EDTA, 62.5 mM NaCl, 25% w/v sucrose, pH 8.0), frozen in a dry ice-ethanol bath, and stored at −80 °C. Chromatin immunoprecipitation-sequencing The frozen B. burgdorferi cells were thawed on ice. One hundred microliters of cells were used to prepare DNA samples for whole genome sequencing (see below), and 400 μL were processed for chromatin immunoprecipitation-sequencing (ChIP-seq) as described previously [99] . Briefly, the fixed cells were lysed using lysozyme at 4 mg/mL final concentration. Crosslinked chromatin was sheared to an average size of 250 bp by sonication using a Qsonica Q800R2 water bath sonicator. The lysate was precleared using Protein A magnetic beads (Fisher 45-002-511) and was then incubated with 4 μL undiluted anti-GFP antibodies [100] or anti-mCherry antibodies [67] overnight at 4˚C. The next day, the lysate was incubated with Protein A magnetic beads for 1 h at 4 °C. After washes and elution, the immunoprecipitate was incubated at 65 °C overnight to reverse the crosslinks. The DNA was next treated with RNase A, proteinase K, extracted with phenol:chloroform:isoamyl alcohol (25:24:1), resuspended in 100 µL of buffer EB (Qiagen), and used for library preparation with the NEBNext UltraII kit (E7645). The library was sequenced using Illumina NextSeq500 at Indiana University’s Center for Genomics and Bioinformatics. Whole genome sequencing For whole genome sequencing (WGS), 100 μL of the frozen cells from above were pelleted, resuspended in 100 µL of TE (50 mM Tris pH 8.0, 10 mM EDTA) containing 1 µL of proteinase inhibitor (Sigma P8340) and 6 µL of Ready-Lyse lysozyme (Epicentre, R1810M), and incubated at 37 °C for 1.5 h. SDS was added to the cell suspension to a final concentration of 1% to solubilize the chromatin. A volume of 150 μL of TES (50 mM Tris pH 8.0, 10 mM EDTA, 1% SDS) was added to the solution and the cell lysate was incubated at 65˚C to reverse the crosslinks. After reversal of crosslinks, the WGS samples were processed and sequenced in the same way as ChIP-seq samples above. WGS of B31-derived strain S9 (see Supplementary Data 1 ) was performed on cells grown and treated similarly to the ones used for the ChIP experiments described above. Strain CJW_Bb523 was grown in 40 mL BSK-II medium to a density of ~3–6 × 10 7 cells/mL. The culture was pelleted at 4000 × g for 10 min in the swinging bucket rotor, resuspended in 1 mL cold HN buffer, and re-pelleted. Genomic DNA was then extracted using DNeasy Blood and Tissue Kits (Qiagen) following the manufacturer’s recommendation for Gram-negative bacteria. Library preparation and whole-genome sequencing were done by the Yale Center for Genome Analysis on a NovaSeq6000 instrument with 2 × 150 bp read length. Sequence mapping and analysis The sequencing reads for ChIP-seq and WGS were mapped using CLC Genomics Workbench (CLC Bio, Qiagen) to the combined B. burgdorferi genome (NCBI GCA_000008685.2_ASM868v2), modified as described below and in Supplementary Data 2 , Worksheet 2. For each strain, the ChIP-seq reads were mapped to a genome sequence carrying the appropriate genetic modifications. Strains CJW_Bb378, CJW_Bb379, CJW_Bb403, CJW_Bb488, CJW_Bb519, CJW_Bb520, CJW_Bb524, CJW_BB525, and CJW_Bb610 have a P flaB - aphI - flaB t kanamycin resistance cassette replacing the intergenic region between parZ and parB . Additionally, they carry a translational fusion to one of the Par proteins, as well as, in some cases, deletion of a par gene. Since the binding of ParB and ParZ fusions to the par locus of these genetically modified strains also involved binding to the P flaB and flaB t sequences inserted into the par locus during strain generation, reads associated with these sequences were erroneously mapped to the endogenous P flaB and flaB t sequences located in the flaB locus. To circumvent this problem, we removed the P flaB and flaB t sequences from the flaB locus of the genome sequences prior to ChIP-seq read mapping. Since these ChIP-seq strains also contain a Δ bbe02 ::P flaB - aadA genetic modification on lp25, we also removed the P flaB sequence from this modified lp25 sequence prior to read mapping. For the same reasons, prior to read mapping, we removed the chromosomal sequences P 0826 and P flgB , in strain CJW_Bb101, which carries P 0826 and P flgB close to the parZ insert on the shuttle vector. Similarly, to prevent erroneous read mapping, we removed the parB sequence from the shuttle vector in strain CJW_Bb403. We note that this shuttle vector lacks a parS site. In the absence of parS , mCherry-ParB is not expected to bind the shuttle vector parB sequence significantly, as evidenced by the absence of fluorescent puncta formation (Supplementary Fig. 1b ). For all ChIP-seq samples, final mapping was done to a concatenated genome sequence obtained by linking the chromosomal sequence, modified as described above, to the sequences of the plasmids present in each strain. Additionally, since shuttle vectors are found in five-fold higher copy number than the chromosome [22] , [23] , [63] , for strains containing shuttle vectors we included 5 tandem copies of the shuttle vector in the concatenated genome prior to read mapping, then summed the binding to these copies. Sequencing reads from each ChIP and WGS samples were normalized by the total number of reads. The WGS results were used as the “input” control for ChIP-seq samples. For marker frequency analysis, the reads corresponding to the oriC and terC regions were averaged over a 30 kilobase span. For the plasmids, the reads were averaged over the entire size of each plasmid. The ChIP enrichment (ChIP/input) and the locus ratios were plotted and analyzed using R scripts, which are available from https://github.com/xindanwanglab/takacs-2022-natcomm [101] . For the whole genome sequencing of strain CJW_Bb523, the sequencing reads were processed using Trimmomatic [102] (parameter = PE, -phred33, -baseout, ILLUMINACLIP:2:30:10, TRAILING:20, MINLEN: 36) and around 8 million reads were mapped to B. burgdorferi B31 genome using Bowtie2 [103] (parameter = -non-deterministic). HTSeq [104] was used to obtain the genomic coverage. The normalized count for each plasmid was calculated as the sum of reads at every base pair (bp) divided by the plasmid size. For oriC , we only considered reads mapped to nucleotide position 443,037-473,267 (~30 kb region, similar to the average size of Borrelia plasmids) on the main chromosome. DNA fluorescence in situ hybridization (FISH) B. burgdorferi cells were washed and resuspended in 1x PBS prior to the FISH experiments in order to remove contaminants from the BSK-H/BSK-II media. Cells were placed on poly-L-lysine coated wells that were outlined on coverslips with a hydrophobic pen (Super PAP pen, Invitrogen #008899). Prior to use, the coverslips were cleaned by sonication steps in 1 M KOH, miliQ water, and 70% ethanol alternated with triple milliQ water rinses, as described previously [41] . Once applied to the poly-L-lysine coated wells, B. burgdorferi cells were fixed in 4% formaldehyde in PBS for 5 min at RT. Cells were then washed 3 times in PBS. Cells were permeabilized using 400 μg/mL lysozyme in GTE buffer (50 mM glucose, 25 mM Tris, 10 mM EDTA, pH 8.0), then washed 3 times with PBS. A hybridization buffer was adapted from a previous report [105] . Briefly, 1 g dextran sulfate was dissolved in 5 mL dH2O, then 3530 μL formamide, 10 mg E. coli tRNA, 1 mL 20× SSC buffer (175.3 g/L NaCl, 88.2 g/L sodium citrate, pH 7.0), and 80 μL of 25 mg/mL BSA were added. The hybridization buffer was filtered and stored at -20 °C. Cells, after fixation and permeabilization, were pre-hybridized in hybridization buffer containing 1 mg/mL RNase A for 30 min. Then, the cells were denatured on a heat block at 94 °C for 5 min. First, the cells were placed on the heat block for 1 min in pre-hybridization solution, which was then replaced with hybridization solution, containing 200 nM probe. The Stellaris locked nucleic acid oligonucleotide FISH probe (sequence 5′-GAATAAGTAAAAGTGGTTTAG-3′, labeled with the dye 6FAM) was synthesized at Biosearch Technologies. This probe recognized a highly repetitive sequence present in 176 copies on plasmid lp21 of strain B31 and in the right subtelomeric region of the chromosome of strain 297 [18] , [106] . The large number of repeats ensured that a strong fluorescent signal could be achieved despite using a single fluorescent probe. Strain B31e2 [107] , which no longer harbors plasmid lp21 of the parental strain B31, served as a negative control as it lacks the target sequence of FISH probe. Hybridization proceeded at RT for 2 h. Wells were then washed as follows: 3 × 10 min washes with 40% (wt/vol) formamide in 2× SSC, 2 × 5 min washes in 2x SSC, and 3× washes in 1× PBS. Prior to imaging, 1 mg/mL DAPI in SlowFade® Gold Antifade Mountant (Thermo Fisher #S36937) was applied to each well. RNA isolation, qRT-PCR, and qPCR For RNA isolation, exponentially growing B. burgdorferi cultures were diluted to 2 × 10 5 cells/mL in 30 mL BSK-II, grown in duplicate for 2 days, then RNA was extracted and quantified as previously described [85] . The cells were pelleted using a 10 min centrifugation at 4300 × g in a swinging bucket rotor. The pellet was resuspended in 400 μL buffer HN [98] (50 mM NaCl, 10 mM HEPES, pH 8.0). RNA was stabilized using the RNAprotect bacteria reagent (Qiagen), extracted using enzymatic lysis and proteinase K digestion (protocol 4 in the RNAprotect bacteria reagent manual), and purified using the RNeasy minikit (Qiagen). DNA was removed using the Turbo DNA-free kit (Thermo Fisher Scientific). RNA was quantified using the Kapa SYBR Fast one-step qRT-PCR mastermix kit (Roche) using 10 ng total RNA per reaction, in duplicate. One additional reaction was performed for each sample without the reverse transcriptase and confirmed that the measured amplification was not due to DNA contamination of the RNA samples. The primers used for amplification of the parZ transcript were 5′-CCCCCTATTTTAAAAACCGAAG-3′ and 5′-TAATGGTTTGCGCGTATCC-3′. The primers used for amplification of the control recA transcript were previously described [19] . The PCR cycling conditions used on a Bio-Rad CFX Connect Real-time system were: reverse transcription (5 min at 42 °C); enzyme activation (5 min at 95 °C); 40 cycles of annealing, extension, and data acquisition (3 sec at 95 °C and 20 s at 60 °C with fluorescence acquisition in the SYBR scan mode); and a melt curve analysis (55 to 95 °C in 0.05 °C increments). The amount of the parZ transcript was normalized to the level of the recA transcript and then expressed for each sample relative to mean levels measured in strain CJW_Bb488 using the ΔΔC T method, as previously described [108] . For the qPCR analysis of genome copy numbers per cell, an exponentially growing culture of strain CJW_Bb339 was diluted to 10 4 cells/mL in triplicate, then culture densities were measured by darkfield counting and samples were harvested at 3, 5, and 7 days. Briefly, 1 mL of culture was centrifuged for 10 min at 10,000 × g and RT. The medium was aspirated and the pellet was resuspended in 1 mL cold buffer HN. The cells were pelleted again for 10 min at 10,000 × g and the pellet was resuspended in 100 μL water, then heat inactivated for 5 min at 99 °C. The volume was brought up to 1 mL by addition of 900 μL of water and the samples were stored at −80 °C. For generation of the standard curves, gBlock DNA fragments identical in sequence to nucleotides 126,973 to 127,294 and 148,101 to 148,426 of the chromosome of B. burgdorferi strain B31 were synthesized at Integrated DNA Technologies. These fragments encompass the sequences amplified by the recA and flaB -specific qPCR primers [19] , [109] , respectively, plus 50 additional bases on each side. The synthesized fragments were resuspended in water to a stock concentration of 10 10 molecules/μL, then 10-fold serial dilutions in water were performed to generate standards of known concentrations. qPCR reactions were set-up using the Kapa SYBR Fast one-step qRT-PCR mastermix kit (Roche) without the reverse transcriptase. A total reaction of 20 μL was setup, which included 1 μL of standard (run in duplicate) or of sample (run in quadruplicate). The PCR conditions were identical to those for the qRT-PCR assay described above except that the reverse transcription step was omitted. DNA concentrations of the samples were calculated based on the standard curve using the CFX Maestro Software (Bio-Rad). Phylogenetic analyses Protein sequences were retrieved from the NCBI databases by Standard Protein BLAST searches using B. burgdorferi proteins as queries in the NCBI BLASTP web-based platform. For Borreliaceae ParZ sequence alignments and phylogenetic tree building and for Brachyspira , Leptospira , and Treponema ParB sequence alignments, only non-redundant RefSeq protein sequences were analyzed. For Leptospira , the analysis of ParB sequences was limited to those encoded by chromosome I. For ParZ-like phylogenetic tree building, all BLAST hits retrieved using B. burgdorferi ParZ as query were utilized. The BLAST search was performed across the three domains of life and among virus sequences. Sequences were aligned and the phylogenetic trees were built using the Geneious R10.0.9 sequence analysis software. Statistics and reproducibility Statistical analyses were performed in GraphPad Prism 9.3.1 software or in Microsoft Excel 365. With the exception of the tick imaging experiment (Fig. 3 ), where one tick was processed for imaging, all other imaging experiments were performed at least twice. The images shown in Figs. 1 a, 1 c, 1 d, 1 f, 2 a, 7 a, 7 b, 7 d, 7 e, 7 f, 7 h, 8 a, 8 b, 8 c, 9 a, 9d and in Supplementary Fig. 1b , 1c , 1d , 1g , 4f , 4g , 6c , 6f are therefore representative of at least two independent imaging instances of the same strain. The images shown in Fig. 4a for strain CJW_Bb474 are representative for that strain, and for strain CJW_Bb379, which was imaged under the same experimental conditions. Strains CJW_Bb474 is derived from strain CJW_Bb379 and expresses free GFP which does not affect the oriC copy number or density (Fig. 1b ). Statistical summaries for all figure panels that involve data quantification are provided in Supplementary Data 2 , Worksheet 3, and include the following information: strain used in the figure, number of imaging samples analyzed, and total number of cells for the combined replicates. Data visualization Data visualization was achieved using the following software: MATLAB R2019a, GraphPad Prism 9.3.1, FiJi [96] , and Adobe Illustrator 2023. Plasmid construction methods Plasmids are listed in Supplementary Data 1 , Worksheet 2. Oligonucleotide primers used in the plasmid generation process are listed in Supplementary Data 1 , Worksheet 3. Requests for the plasmids generated in this study should be directed to Christine Jacobs-Wagner. I. Shuttle vectors pBSV2G_P 0826 -mCherry Bb -ParB The following fragments were assembled (using intermediary constructs) between the SacI and PstI sites of plasmid pBSV2G_2: (a) the promoter of B. burgdorferi gene bb0826 (P 0826 ) [89] , corresponding to bp 535523-535703 of strain B31’s chromosome, PCR-amplified with primers NT115 and NT116 and digested with SacI and BamHI; (b) the mcherry Bb sequence [89] , amplified with primers NT100 and NT101 and digested with KpnI and BamHI; (c) parB ( bb0434 ), amplified from strain B31’s genomic DNA with primers NT230 and NT232 and digested with SalI and PstI. pBSV2G_P 0826 -RBS-ParZ-msfGFP Bb The following fragments were assembled (using intermediary constructs) between the SacI and KpnI and between the PstI and HindIII sites of plasmid pBSV2G_2, respectively: (a) promoter P 0826 [89] , flanked by SacI and BamHI restriction enzyme sites; (b) parZ ( bb0432 ), PCR-amplified from strain B31’s genomic DNA with primers NT363 and NT364 and digested with BamHI and KpnI; (c) the msfgfp Bb sequence [89] , PCR-amplified with primers NT159 and NT160 and digested with PstI and HindIII. pKFSS1_P 0826 -mCherry Bb -ParB P 0826 - mcherry Bb - parB was moved from pBSV2G_P 0826 -mCherry Bb -ParB into pKFSS1_2 using SacI and HindIII. pKFSS1_P 0826 -msfGFP Bb -ParB msfgfp Bb was PCR amplified using primers NT341 and NT162, digested with BamHI and KpnI and ligated into the BamHI/KpnI backbone of pKFSS1_P 0826 -mCherry Bb -ParB. pBSV2G_P 0031 -mCherry Bb -ParB P1 The following fragments were assembled, through intermediates, between the SacI/KpnI, and XbaI/HindIII sites of pBSV2G_2: promoter P 0031 [89] , obtained from strain B31’s genomic DNA by amplification with primers NT111 and NT112 and digestion with SacI and BamHI; mcherry Bb , PCR amplified with NT100 and NT101 and digested with BamHI and KpnI; and parB P1 , obtained by de novo gene synthesis at Genewiz flanked by XbaI and HindIII restriction enzyme sites. The parB P1 gene encodes the P1 plasmid ParB protein minus its N-terminal peptide sequence (ParB ΔN30 ) [110] , which was codon-optimized for translation in B. burgdorferi using the web-based JAVA Codon Adaptation tool hosted at www.jcat.de [111] as previously described [89] and was deposited at GenBank under accession number ON321895. pBSV2G_P 0031 -msfGFP Bb -ParB P1 msfgfp Bb was PCR amplified using primers NT161 and NT162, digested with BamHI and KpnI, and cloned into the BamHI/KpnI sites of pBSV2G_P 0031 -mCherry Bb -ParB P1 . pBSV2B_P 0826 -mCherry Bb -ParB P 0826 - mcherry Bb - parB was moved from pBSV2G_P 0826 -mCherry Bb -ParB into pBSV2B using SacI and HindIII digestion. pBSV2B_r(P 0031 -msfGFP Bb -ParB P1 )_P 0826 -mCherry Bb -ParB P 0031 - msfgfp Bb - parB P1 was released from pBSV2G_P 0031 -msfGFP Bb -ParB P1 as a SacI/FspI fragment and was ligated into the SacI/BsrBI backbone of pBSV2B_P 0826 -mCherry Bb -ParB. pBSV2G_P smcL -mCherry Bb -Smc The following fragments were sequentially assembled within the multicloning site of plasmid pBSV2G_2: mcherry Bb , PCR-amplified using primers NT100 and NT101 and digested with BamHI and KpnI; a DNA fragment of 804 bp upstream of the ttg START codon of smc ( bb0045 ), PCR - amplified with primers NT217 and NT219 and digested with SacI and BamHI; and a DNA fragment encoding smc ( bb0045 ), PCR-amplified using primers NT221 and NT222 and digested with SalI and PstI. pBSV2G_P 0826 -ParA-msfGFP Bb The following fragments were assembled between the SacI and HindIII sites of pBSV2G_2: (i) promoter P 0826 [89] , flanked by SacI and BamHI restriction enzyme sites; (ii) msfGFP Bb , obtained by PCR amplification using primers NT159 and NT160 and flanked by PstI and HindIII restriction enzyme sites; and parA ( bb0431 ), obtained by PCR amplification using primers NT345 and NT226 and digestion with BamHI and KpnI. pBSV2H_P 0826 -ParA-msfGFP Bb P 0826 -ParA-msfGFP Bb was transferred from pBSV2G_P 0826 -ParA-msfGFP Bb into pBSV2H using BsrBI and AvrII. II. Suicide vectors Note on nomenclature: “pKI” signifies a suicide vector generated to mediate knock-in of a gene of interest into the B. burgdorferi genome. While most of these plasmids are based on pCR2.1, some are based on other backbones. The antibiotic resistance used for selection is noted in the name of the construct (i.e. pKIKan, pKIGent, or pKIStrep) and is driven by default by the P flgB promoter. When, instead, the P flaB promoter was used to drive antibiotic resistance gene expression, this is noted in the name of the plasmid (e.g., pKIKan(P flaB )). pKIGent This plasmid, obtained through a series of intermediate constructs, contains the following features: a) a Δ aphI Δ bla backbone of plasmid pCR2.1 [85] , flanked by HindIII and XbaI restriction enzyme sites; b) a P flgB - aacC1 - flaB t cassette flanked by SpeI and SacII restriction enzyme sites. This cassette is flanked by two multicloning sites, namely HindIII-KpnI-SacI-BamHI-SpeI-XmaI and SacII-EcoRI-PstI-NotI-XhoI-SphI-XbaI. To generate this cassette, the following fragments were assembled through intermediates: (i) P flgB - aacC1 [87] was cloned in between the XmaI and the SacII sites of the backbone; (iii) flaB t, the flagellin transcriptional terminator, was generated by annealing primers NT350 and NT351 and ligating them into the SpeI/XmaI sites of the backbone. This inactivated the original XmaI site of the backbone but generated a new one downstream of flaB t. pKIGent_parS P1 This plasmid differs from pKIGent, in that the parS P1 sequence [112] was synthesized de novo at Genewiz and cloned into the pUC57Amp backbone. It was then PCR-amplified using primers NT165 and NT166, digested with SpeI and XmaI, and inserted into the SpeI/XmaI sites of the backbone. The resulting clone had a mutation in the parS P1 sequence that was corrected by site-directed mutagenesis using primers NT215 and NT216. pKIGent_parS P1 _phoU B. burgdorferi B31 chromosomal region from nucleotide 38650 to 40720 was PCR-amplified with primers NT175 and NT176 and digested with SacI and SpeI. The chromosomal region from nucleotide 40721 to 42797 was PCR-amplified with primers NT177 and NT178 and digested with PstI and XhoI. The two fragments were inserted into the SacI/SpeI and PstI/XhoI sites of pKIGent_parS P1 , respectively. pKIGent_parS P1 _cp26 B. burgdorferi B31 cp26 region from nucleotide 20585 to 22602 was PCR-amplified with primers NT203 and NT204 and digested with SacI and BamHI. The cp26 region from nucleotide 22603 to 24632 was PCR-amplified with primers NT205 and NT206 and digested with PstI and XhoI. The two fragments were inserted into the SacI/BamHI and PstI/XhoI sites of pKIGent_parS P1 , respectively. pKIGent_parS P1 _uvrC B. burgdorfe ri strain B31’s chromosomal region from nucleotide 474180 to 476218 was PCR-amplified with primers NT267 and NT268 and digested with SacI and SpeI. The region from nucleotide 476251 to 478279 was PCR-amplified with primers NT269 and NT270 and digested with PstI and XhoI. The two fragments were inserted into the SacI/SpeI and PstI/XhoI sites of pKIGent_parS P1 , respectively. pΔparBS B. burgdorferi chromosomal region between nucleotides 448842 and 450913 was PCR-amplified with primers NJ99 and NJ100 and digested with BamHI and XmaI. The region from nucleotide 452017 to 453998 was PCR-amplified using primers NJ97 and NJ98 and digested with PstI and XhoI. The two fragments were inserted into the BamHI/XmaI and PstI/XhoI sites of pKIGent, respectively. pΔparBS(Kan) The P flaB -aphI cassette from pKIKan(P flaB ) was excised using PstI and XmaI and inserted into the PstI/XmaI sites of pΔparBS. pKIGent_par The B. burgdorferi chromosomal region from nucleotide 448842 to 450913 was PCR-amplified with primers NJ99 and NJ100 and digested with BamHI and XmaI. 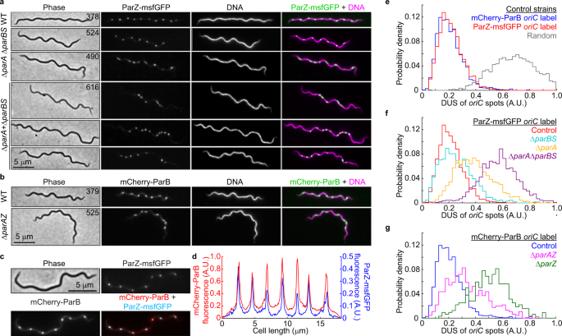Fig. 8: ParZ is a novel bacterial centromere-binding protein that contributes tooriCsegregation. aImages of ParZ-msfGFP signal in strains carrying the full complement ofB. burgdorferi pargenes (WT) or lacking thepargenes and/orparSsequence as indicated. DNA was stained with Hoechst 33342. CJW_Bb strain numbers are listed on the phase-contrast images.bImages of mCherry-ParB signal in strains carrying the full complement ofpargenes (WT) or lacking theparAZoperon, as indicated. DNA was stained with Hoechst 33342. CJW_Bb strain numbers are listed on the phase contrast images.cImages of strain CJW_Bb403 showing colocalization of ParZ-msfGFP and mCherry-ParB signals.dFluorescence intensity profile along the cell length for the cell shown in (c).eHistograms showing the distributions of deviations from uniform spacing (DUS, see methods) oforiCspots in control strains expressing mCherry-ParB (strain CJW_Bb379) or ParZ-msfGFP (strain CJW_Bb378) to labeloriC. Also shown in gray are DUS values obtained by simulating a random redistribution oforiCloci in the analyzed cells of strain CJW_Bb379 (see methods).fHistograms comparing DUS distributions of ParZ-msfGFP-labeledoriCfoci in control (CJW_Bb378), ΔparBS(CJW_Bb524), ΔparA(CJW_Bb490), and ΔparAΔparBS(CJW_Bb616) strains.gHistograms comparing DUS distributions of mCherry-ParB-labeledoriCfoci in control (CJW_Bb379), ΔparAZ(CJW_Bb525), and ΔparZ(CJW_Bb626) strains. Source data for panels (e–g) are provided as a Source Data file. The numbers (n) of cells analyzed and the number of replicates are provided in Supplementary Data2. 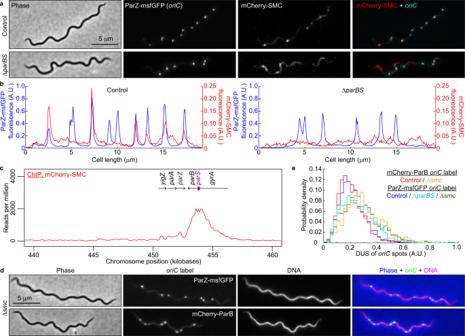Fig. 9: SMC is recruited to theoriCregion by ParB and mildly contributes to regularoriCspacing. aImages of cells expressing ParZ-msfGFP (to labeloriC) and mCherry-SMC in control (CJW_Bb602, carrying the full complement ofpargenes) and ΔparBS(CJW_Bb615) strains.bFluorescence intensity profiles along the cell length for the cells shown in (a).cChIP-seq profile showing the binding of mCherry-SMC to theparlocus in strain CJW_Bb601. Genes underlining the enriched sequence reads are highlighted.dImages of cells showingoriClocalization in Δsmcstrains in which theoriCis labeled with either ParZ-msfGFP (CJW_Bb603) or mCherry-ParB (CJW_Bb604). Hoechst 33342 was used to stain the DNA. An overlay is also shown.eHistograms showing DUS oforiCspots in cells of control and Δsmcstrains in whichoriCwas labeled with either ParZ-msfGFP (control, CJW_Bb378; Δsmc, CJW_Bb603) or mCherry-ParB (control, CJW_Bb379; Δsmc, CJW_Bb604). Also shown is the DUS histogram for the ΔparBSstrain CJW_Bb524. Source data are provided as a Source Data file. The numbers (n) of cells analyzed and the number of replicates are provided in Supplementary Data2. The region between nucleotides 451133 and 453037 was PCR-amplified with primers NJ101 and NJ102 and digested with PstI and XhoI. The two fragments were inserted into the BamHI/XmaI and PstI/XhoI sites of pKIGent, respectively. pKIGent_parS P1 _lp17 The 1.3 kilobase pair (kbp) BamHI/FspI fragment of pKIGent_parS P1 was ligated with the 2.9 kbp BamHI/NaeI backbone of pKK81. pΔparAZ Nucleotides 447274 through 449320 of strain B31 chromosome were PCR-amplified using primers NT530 and NT531, digested with BamHI and XmaI, and ligated into the BamHI/XmaI backbone of pKIGent_par. pΔparZ Nucleotides 448134 through 450172 of the B31 chromosome were PCR-amplified using primers NT528 and NT529, cut with BamHI and XmaI, and ligated into the BamHI/XmaI backbone of pKIGent_par. pΔparAZBS Nucleotides 447274 through 449320 of the B31 chromosome were PCR-amplified using primers NT530 and NT531, digested with BamHI and XmaI, and ligated into the BamHI/XmaI backbone of pΔparBS. pKIGent_parS P1 _lp28-3 Nucleotides 1853 to 3891 of plasmid lp28-3 were PCR-amplified using primers NT487 and NT488 and digested with KpnI and BamHI. Nucleotides 3890 to 5944 of plasmid lp28-3 were PCR-amplified using primers NT489 and NT490 and digested with SacII and XhoI. These fragments were cloned into the corresponding sites of pKIGent_parS P1 . pKIGent_parS P1 _lp28-2 Plasmid lp28-2 was PCR-amplified using primers NT483 and NT484 and digested with KpnI and SpeI. Plasmid lp28-2 was PCR-amplified using primers NT485 and NT486 and digested with SacII and XhoI. These fragments were cloned into the corresponding sites of pKIGent_parS P1 . pKIGent_parS P1 _lp25 The P flgB - aacC1 - parS P1 cassette was PCR-amplified from pKIGent_parS P1 using primers NT509 and NT524, cut with PacI and MluI, and cloned into the PacI/MluI backbone of pKbeKan. pKIGent_parS P1 _lp38 Nucleotides 20973 through 23014 of plasmid lp38 were PCR-amplified using primers NT499 and NT500, then digested with KpnI and SpeI. Nucleotides 23014 through 25091 of plasmid lp38 were PCR-amplified using primers NT501 and NT502, then digested with SacII and XhoI. The fragments were ligated into the corresponding sites of pKIGent_parS P1 . pKIGent_parS P1 _lp36 Plasmid lp36 was PCR-amplified with primers NT495 and NT496, digested with KpnI and BamHI, then cloned into the KpnI/BamHI sites of pKIGent_parS P1 . The resulting plasmid was PCR-amplified using primers MRS_17 and MRS_18 and Gibson-assembled with a PCR product obtained by amplification of plasmid lp36 using primers MRS_19 and MRS_20. pKIKan This plasmid was obtained through a series of intermediate constructs, and in a manner similar to pKIGent, except that is has an aphI kanamycin resistance gene instead of an aacC1 gentamicin resistance gene under the control of P flgB . It contains the following features: a) the Δ aphI Δ bla backbone of plasmid pCR2.1 [85] , flanked by HindIII and XbaI restriction enzyme sites; b) a P flgB - aphI - flaB t cassette flanked by SpeI and SacII restriction enzyme sites that are part of two multicloning sites: HindIII-KpnI-SacI-BamHI-SpeI-XmaI and SacII-PstI-NotI-XhoI-SphI-XbaI. To generate this cassette, the following fragments were assembled through intermediates: (i) P flgB , flanked by SacII and NdeI sites; (ii) aphI , PCR-amplified from pBSV2 using primers NT534 and NT535, digested with NdeI and XmaI, and cloned together with P flgB between the SacII and XmaI sites of the backbone; and (iii) flaB t, generated by annealing primers NT350 and NT351 and ligating them into the SpeI/XmaI sites of the backbone. This inactivated the original XmaI site of the backbone but generated a new one downstream of flaB t. pKIKan(P flaB ) P flaB was PCR-amplified from pBSV2G_P flaB -mCerulean Bb using primers NT577 and NT578, digested with SacII and NdeI, and ligated into the SacII/NdeI backbone of pKIKan. pKIKan_parS P1 P flgB - aphI-flaB t was moved from pKIKan into the backbone of pKIGent_parS P1 as an XmaI/PstI fragment. pKIKan(P flaB )_parS P1 The P flaB - aphI - flaB t cassette was moved from pKIKan(P flaB ) into the backbone of pKIGent_parS P1 as an XmaI/PstI fragment. pKIKan_parS P1 _uvrC P flgB - aphI - parS P1 was excised from pKIKan_parS P1 using SpeI and PstI and inserted into the SpeI/PstI backbone of pKIGent_parS P1 _uvrC, where it replaced P flgB - aacC1 - parS P1 . pKIGent_parS P1 _lp28-4 The pKIGent_parS P1 backbone was PCR-amplified using primers MRS_46 and MRS_31. Plasmid lp28-4 was PCR-amplified using primers MRS_49 and MRS_53, and MRS_51 and MRS_52, respectively. The P flgB - aacC1 - parS P1 cassette was PCR-amplified from pKIGent_parS P1 using primers MRS_32 and MRS_33. The four PCR products were Gibson assembled together. pKIGent_parS P1 _lp54 pABA01 was PCR-amplified using primers MRS_24 and MRS_29. The P flgB - aacC1 - parS P1 cassette was PCR-amplified from pKIGent_parS P1 using primers MRS_25 and MRS_26. The two PCR products were Gibson assembled. pΔparS A region between nucleotides 449961 and 451998 of strain B31’s chromosome was PCR-amplified using primers NT625 and NT626, digested with BamHI and XmaI, and inserted into the BamHI/XmaI sites of plasmid pΔparBS. pΔparB A region from nucleotide 451996 to nucleotide 453998 of strain B31’s chromosome was PCR amplified using primers NT627 and NT628, digested with PstI and XhoI, and inserted into the PstI/XhoI sites of pΔparBS. pΔparA(Kan) parA was deleted from pKIKan(P flaB )_par by site-directed mutagenesis using primers NT623 and NT624. pKIKan(P flaB )_par The P flaB -aphI-flaB t cassette from pKIKan(P flaB ) was excised using PstI and XmaI and inserted into the PstI/XmaI sites of pKIGent_par. pKIKan(P flaB )_ParZ-msfGFP Bb msfgfp Bb was PCR-amplified with primers NT643 and NT644. Plasmid pKIKan(P flaB )_par was PCR-amplified with primers NT645 and NT646. The two fragments were Gibson-assembled. pKIKan(P flaB )_mCherry Bb -ParB mcherry Bb was PCR-amplified with primers NT629 and NT630. Plasmid pKIKan(P flaB )_par was PCR-amplified with primers NT631 and NT632. The two fragments were Gibson-assembled. pKIGent_parS P1 _lp28-1 P flgB -aacC1_parS P1 was PCR-amplified from pKIGent_parS P1 using primers NT762 and NT763. The backbone of p28-1::flgBp-aacC1 was PCR-amplified using primers NT764 and NT765. The two fragments were Gibson-assembled together. pKIKan(P flaB )_ParA-msfGFP Bb msfgfp Bb was PCR-amplified using primers NT633 and NT634. parA was PCR-amplified using primers NT636 and NT768. parZ was PCR-amplified from pKIKan(P flaB )_par using primers NT766 and NT635. The suicide vector backbone was PCR-amplified from pKIKan(P flaB )_par using primers NT769 and NT767. The four PCR products were Gibson-assembled together. pKIKan(P flaB )_ParZ-msfGFP Bb _ΔparA Site-directed mutagenesis was performed on plasmid pKIKan(P flaB )_ParZ-msfGFP Bb using primers NT623 and NT624. pKIKan(P flaB )_ParA-msfGFP Bb _ΔparZ Site-directed mutagenesis was performed on plasmid pKIKan(P flaB )_ParA-msfGFP Bb using primers NT778 and NT779. pKIKan(P flaB )_ΔparBS_ParA-msfGFP Bb The BamHI/XmaI insert of plasmid pKIKan(P flaB )_ParA-msfGFP Bb was ligated into the BamHI/XmaI backbone of plasmid pΔparBS(Kan). pKIKan(P flaB )_ΔparBS_ParZ-msfGFP Bb The BamHI/XmaI insert of plasmid pKIKan(P flaB )_ParZ-msfGFP Bb was ligated into the BamHI/XmaI backbone of plasmid pΔparBS(Kan). pKIKan(P flaB )_mCherry Bb -ParB_ΔparAZ The BamHI/XmaI insert of plasmid pΔparAZ was ligated into the BamHI/XmaI backbone of plasmid pKIKan(P flaB )_mCherry Bb -ParB. pKIKan(P flaB )_ParA-msfGFP Bb _ParZ ΔN20 Site-directed mutagenesis was performed on pKIKan(P flaB )_ParA-msfGFP Bb using primers NT1020 and NT1021. pKIGent_parS P1 _lp21_V2 The backbone of pKIGent_parS P1 was PCR-amplified with primers NT800 and NT801. The P flgB -aacC1_parS P1 cassette was PCR-amplified from pKIGent_parS P1 with primers NT796 and NT797. Nucleotides 253 through 1114 of the B31 plasmid lp21 were PCR-amplified using primers NT794 and NT795. Nucleotides 1115 through 2628 of the B31 plasmid lp21 were PCR-amplified using primers NT798 and NT799. The four PCR products were Gibson-assembled. pKIGent_parS P1 _lptD The backbone of pKIGent_parS P1 was PCR-amplified with primers NT824 and NT825. The P flgB -aacC1_parS P1 cassette was PCR-amplified from pKIGent_parS P1 with primers NT820 and NT821. Nucleotides 895077 through 896572 of the B31 chromosome were PCR-amplified using primers NT818 and NT819. Nucleotides 896573 through 898070 of the B31 chromosome were PCR-amplified using primers NT822 and NT823. The four PCR products were Gibson-assembled. pKIGent_mCherry Bb -Smc The following fragments were Gibson-assembled: 1) nucleotides 43811 through 45353 of the B31 chromosome fused downstream of and in frame to mcherry Bb , controlled by the smc native promoter, obtained by PCR-amplification of plasmid pBSV2G_P smcL -mCherry Bb -Smc with primers NT1006 and NT1007; 2) the gentamicin cassette of pKIGent_parS P1 _phoU, obtained by PCR-amplification with primers NT1008 and NT1009; 3) nucleotides 45376 through 46530 of the B31 chromosome, obtained by PCR-amplification with primers NT1010 and NT1011; and 4) the suicide vector backbone of plasmid pΔparA(kan), obtained by PCR-amplification with primers NT1012 and NT1013. pΔsmc(gent) The following fragments were Gibson-assembled: 1) nucleotides 42016 through 43530 of the B31 chromosome, obtained by PCR amplification with primers NT960 and NT961; 2) the gentamicin cassette of pKIGent_parS P1 _phoU, obtained by PCR amplification with primers NT962 and NT963; 3) nucleotides 45332 through 46857 of the B31 chromosome, obtained by PCR amplification with primers NT964 and NT965; and 4) the suicide vector backbone of plasmid pΔparA(kan), obtained by PCR amplification with primers NT966 and NT967. pKIGent_ΔparBS_ParZ-msfGFP Bb _ΔparA The gentamicin resistance cassette was excised from pΔparB as a SacII/XmaI fragment and inserted into the SacII/XmaI backbone of plasmid pKIKan(P flaB )_ΔparBS_ParZ-msfGFP Bb _ΔparA. pKIKan(P flaB )_ΔparBS_ParZ-msfGFP Bb _ΔparA The BamHI/XmaI insert of plasmid pKIKan(P flaB )_ParZ-msfGFP Bb _ΔparA was ligated into the BamHI/XmaI backbone of plasmid pΔparBS(Kan). pKIKan(P flaB )_mCherry Bb -ParB_ΔparZ The BamHI/XmaI insert of plasmid pΔparZ(Kan) was ligated into the BamHI/XmaI backbone of plasmid pKIKan(P flaB )_mCherry Bb -ParB. pΔparZ(Kan) The P flaB - aphI cassette of pKIKan(P flaB ) was excised using PstI and XmaI and ligated to the PstI/XmaI backbone of plasmid pΔparZ. pKIStrep(P flaB )_parS P1 aadA was PCR-amplified from pJSB252 using with primers NT756 and NT757. The backbone of the pKIKan(P flaB )_parS P1 plasmid was PCR-amplified using primers NT758 and NT759. The two fragments were Gibson-assembled with each other. pKIStrep_parS P1 _Tn pGKT was digested with EagI, and the resulting 1.8 kbp fragment was purified and ligated, yielding plasmid pTG, which was then PCR-amplified using primers NT690 and NT691. P flaB - aadA _ parS P1 was PCR-amplified from pKIStrep(P flaB )_parS P1 using primers NT692 and NT693. The two PCR products were Gibson assembled with each other. The resulting plasmid was PCR amplified with NT784 and NT785 and the resulting PCR product was digested with AvrII and self-ligated. Reporting summary Further information on research design is available in the Nature Portfolio Reporting Summary linked to this article.